Orexin neurons inhibit sleep to promote arousal Humans and animals lacking orexin neurons exhibit daytime sleepiness, sleep attacks, and state instability. While the circuit basis by which orexin neurons contribute to consolidated wakefulness remains unclear, existing models posit that orexin neurons provide their wake-stabilizing influence by exerting excitatory tone on other brain arousal nodes. Here we show using in vivo optogenetics, in vitro optogenetic-based circuit mapping, and single-cell transcriptomics that orexin neurons also contribute to arousal maintenance through indirect inhibition of sleep-promoting neurons of the ventrolateral preoptic nucleus. Activation of this subcortical circuit rapidly drives wakefulness from sleep by differentially modulating the activity of ventrolateral preoptic neurons. We further identify and characterize a feedforward circuit through which orexin (and co-released glutamate) acts to indirectly target and inhibit sleep-promoting ventrolateral preoptic neurons to produce arousal. This revealed circuitry provides an alternate framework for understanding how orexin neurons contribute to the maintenance of consolidated wakefulness and stabilize behavioral state. Orexin (Ox; also called hypocretin) neurons in the lateral hypothalamus play an indispensable role in stabilizing and maintaining wakefulness. For example, loss of Ox- producing neurons in people with narcolepsy, results in debilitating excessive daytime sleepiness, sleep attacks, and wake-instability [1] . The narcoleptic phenotype is nearly fully recapitulated in Ox-deficient animal models [2] , [3] , [4] . While existing circuit models hold that Ox neurons stabilize wake by exciting other brain arousal nodes, —for example, Ox neurons increase wake by exciting noradrenergic locus coeruleus neurons [5] , we hypothesized here that Ox neurons may instead (or also) produce their wake-promoting and wake-stabilizing effects through inhibition of neurons of the ventrolateral preoptic nucleus (VLPO), a region that is essential for initiating and maintaining sleep. The cellular VLPO contains neurons that are active during sleep, lesions of the VLPO result in profound and persisting insomnia, and acute stimulation of the VLPO, in particular resident GABA/galanin-containing VLPO neurons (VLPO GABA/Gal ), produces sleep [6] , [7] , [8] , [9] , [10] . Local administration of Ox into the VLPO also rouses animals from sleep, although how Ox acts on its postsynaptic cellular targets, and the identity of these targets, within the VLPO remains unresolved [11] . Given that Ox is an excitatory peptide, and that Ox neurons co-release glutamate, we predicted that Ox/glutamate input would not produce arousal by directly inhibiting sleep-promoting VLPO GABA/Gal neurons, as some other arousal inputs to the VLPO appear to do [12] , [13] , but rather would inhibit VLPO GABA/Gal neurons indirectly. Ox might, for example, inhibit VLPO GABA/Gal neurons by activating a GABAergic afferent input to the VLPO, or do so via an additional, inhibitory synaptic relay. We hypothesized that Ox regulation of arousal depends upon a polysynaptic pathway from the lateral hypothalamus to an intra- VLPO circuit that comprises Ox-responsive GABAergic (VLPO GABA ) interneurons whose collaterals inhibit sleep-promoting VLPO GABA/Gal neurons to produce arousal. To test our hypothesis, we first sought to determine if acute activation of presynaptic Ox inputs (Ox terminals) within the VLPO could trigger behavioral and electroencephalographic arousal from sleep. We then employed in vitro pharmacology, optogenetically-based circuit mapping, combined with single-cell transcriptomics, to determine the neurochemical and molecular phenotypes of the postsynaptic cellular targets of Ox input within the VLPO. In our final experimental step, we sought to identify and characterize the intra-VLPO circuitry and synaptic mechanisms through which Ox inputs to the VLPO might promote and support arousal. In this work, our findings identify a polysynaptic circuit, including an intra-VLPO inhibitory feedforward circuit, through which Ox signaling can rapidly produce, and maintain, arousal. In vivo stimulation of orexin terminals in the VLPO rapidly triggers arousals from both NREM and REM sleep Orexin neurons innervate the preoptic region including the VLPO [14] , [15] , [16] (Fig. 1a ). We first sought to determine whether activation of Ox terminals in the VLPO could produce or otherwise trigger arousal from sleep. To do so, we injected AAV-DIO-ChR2-mCherry or AAV-DIO-ChR2-eYFP into the Ox field of Ox-IRES-Cre mice and then optogenetically stimulated ChR2(+) Ox terminals in the VLPO in vivo, during both NREM and REM sleep. (Fig. 1 ). Selective expression of mCherry or YFP in Ox neurons was confirmed by double immunofluorescence labeling (Fig. 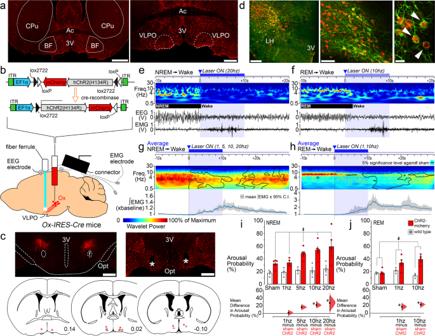Fig. 1: Optogenetic stimulation of orexin terminals in the VLPO rapidly triggers arousals from both NREM and REM sleep. aOrexin innervation of the POA and VLPO (scale bars: 1 and 0.5  mm).bAAV-DIO-ChR2-mCherrywas injected bilaterally into the Ox field ofOx-IRES-Cremice and optical fibers bilaterally placed above the VLPO.cOrexin neurons transduced with ChR2- mCherry (red; left) and optical fiber (*) above the VLPO (right; scale bars: 500  µm). Optical fiber placements (red * ChR2-mCherry and grey * WT; bottom).dChR2-eYFP(+) neurons double-labeled for Ox-A (in red; scale bars: 200; 100, and 20  µm). Laser-induced arousals from NREM (e) and REM (f) sleep (10  s-long periods before and after 10  s light pulses, top). EMG and EEG recordings and continuous EEG wavelet transforms (bottom). Trial-averaged responses to laser stimulation in NREM (g) and REM (h) sleep. EEG wavelet power for trials containing arousals (top;n= 5). Black contour lines: 5% significance level against sham trials (paired bootstrap confidence interval of the mean wavelet power difference). EMG mean responses (grey region: 95% bootstrap confidence interval; bottom). Mean differences in arousal probability, from NREM (i) and REM sleep (j) in ChR2-mCherry (n=  5) and WT (n=  3; top). On the bottom, the mean differences in arousal probability (stimulation vs. sham) within the ChR2-mCherry group (NREM: effect of genotypeF(1, 24)=  22.92,p=  0.003; interaction between genotype and stimulation frequencyF(4, 24)=  1.66,p=  0.192, two-way ANOVA one-repeated-measure. REM: interaction between genotype and stimulation frequencyF(2, 12)=  7.02,p=  0.010, two-way ANOVA one-repeated-measure). Mean difference in arousal probability from NREM (i, bottom;t=  2.98 and 3.73,p=  0.019 and 0.004 for 10 and 20  Hz stimulations) and REM sleep (j, bottom;t=  3.82 and 5.16,p=  0.002 and 0.0007 for 1 and 10  Hz stimulations; post-hoc Holm–Šidákt-tests, two-way ANOVA one-repeated-measure;n=  5; Source Data file). Error bars: SEM; ‡: significant for factor genotype (two-way ANOVA); #, significant interaction between the factors genotype and stimulation frequency (two-way ANOVA). Mean differences (stimulations vs sham within the ChR2-mcherry group) plotted as bootstrap sampling distributions (bottom). Dots: mean difference in arousal probability; vertical error bars: 95% confidence intervals; *p<  0.05 post-hoc Holm–Šidákt-test. All testing was two-tailed, andnrefers to the number of independent animals. 3V 3rdventricle, Opt optic tract, f fornix, Ac anterior commissure, CPu corpus striatum, BF basal forebrain and LH lateral hypothalamus. Atlas levels are per Franklin and Paxinos, 2001. 1d and Supplementary Table 1 ). On average, photostimulation of the Ox terminals in the VLPO consistently produced short-latency arousals during both NREM (Fig. 1e and g ) and REM sleep (Fig. 1 f and h), an effect not seen in sham trials ( n = 5; paired bootstrapping, p > 0.05). When stimulated during NREM sleep, we found that arousal probability in the ChR2-mCherry group ( n = 5) was elevated above that in the wildtype group (WT; n = 3) for all stimulation levels (significant main effect of genotype F (1, 24) = 22.92, p = 0.003; non-significant interaction between genotype and stimulation frequency F (4, 24) = 1.66, p = 0.192, two-way ANOVA; Fig. 1i , top ). However, the significant increases in arousal probability from NREM sleep were observed only during 10 and 20 Hz stimulations ( t = 2.98 and 3.73, p = 0.019 and 0.004, respectively; post-hoc Holm-Šidák t -tests), not at the 1 and 5 Hz stimulation levels ( t = 0.20 and 2.20, p = 0.842 and 0.073, respectively; post-hoc Holm-Šidák t -tests; n = 5). Comparison of the bootstrap confidence intervals and effect sizes at different stimulation frequencies revealed that the effect of 5 Hz stimulation was consistent with the effects of 10 and 20 Hz stimulations but inconsistent with the non-effect at the 1 Hz level (Fig. 1i , bottom ). When stimulation was applied during REM sleep (interaction between genotype and stimulation frequency F ( 2, 12 ) = 7.02, p = 0.010, two-way ANOVA one-repeated-measure; Fig. 1j , top ), arousal probability increased significantly in association with both the 1 and 10 Hz stimulations ( t = 3.82 and 5.16, p = 0.002 and <0.001, respectively; sham versus 1 and 10 Hz conditions within the ChR2-mCherry group, post-hoc Holm- Šidák t -tests; n = 5; Fig. 1j , bottom ). Interestingly, the arousal response during REM sleep appears to be specific to the Ox input to the VLPO given that similar optogenetic stimulation of GABAergic terminals, also arising from the lateral hypothalamic region, in the VLPO rouses mice from NREM but not REM sleep [13] . Fig. 1: Optogenetic stimulation of orexin terminals in the VLPO rapidly triggers arousals from both NREM and REM sleep. a Orexin innervation of the POA and VLPO (scale bars: 1 and 0.5  mm). b AAV-DIO-ChR2-mCherry was injected bilaterally into the Ox field of Ox-IRES-Cre mice and optical fibers bilaterally placed above the VLPO. c Orexin neurons transduced with ChR2- mCherry (red; left) and optical fiber (*) above the VLPO (right; scale bars: 500  µm). Optical fiber placements (red * ChR2-mCherry and grey * WT; bottom). d ChR2-eYFP(+) neurons double-labeled for Ox-A (in red; scale bars: 200; 100, and 20  µm). Laser-induced arousals from NREM ( e ) and REM ( f ) sleep (10  s-long periods before and after 10  s light pulses, top). EMG and EEG recordings and continuous EEG wavelet transforms (bottom). Trial-averaged responses to laser stimulation in NREM ( g ) and REM ( h ) sleep. EEG wavelet power for trials containing arousals (top; n = 5). Black contour lines: 5% significance level against sham trials (paired bootstrap confidence interval of the mean wavelet power difference). EMG mean responses (grey region: 95% bootstrap confidence interval; bottom). Mean differences in arousal probability, from NREM ( i ) and REM sleep ( j ) in ChR2-mCherry ( n =  5) and WT ( n =  3; top). On the bottom, the mean differences in arousal probability (stimulation vs. sham) within the ChR2-mCherry group (NREM: effect of genotype F (1, 24) =  22.92, p =  0.003; interaction between genotype and stimulation frequency F (4, 24) =  1.66, p =  0.192, two-way ANOVA one-repeated-measure. REM: interaction between genotype and stimulation frequency F (2, 12) =  7.02, p =  0.010, two-way ANOVA one-repeated-measure). Mean difference in arousal probability from NREM ( i , bottom; t =  2.98 and 3.73, p =  0.019 and 0.004 for 10 and 20  Hz stimulations) and REM sleep ( j , bottom; t =  3.82 and 5.16, p =  0.002 and 0.0007 for 1 and 10  Hz stimulations; post-hoc Holm–Šidák t -tests, two-way ANOVA one-repeated-measure; n =  5; Source Data file). Error bars: SEM; ‡: significant for factor genotype (two-way ANOVA); #, significant interaction between the factors genotype and stimulation frequency (two-way ANOVA). Mean differences (stimulations vs sham within the ChR2-mcherry group) plotted as bootstrap sampling distributions (bottom). Dots: mean difference in arousal probability; vertical error bars: 95% confidence intervals; * p <  0.05 post-hoc Holm–Šidák t -test. All testing was two-tailed, and n refers to the number of independent animals. 3V 3 rd ventricle, Opt optic tract, f fornix, Ac anterior commissure, CPu corpus striatum, BF basal forebrain and LH lateral hypothalamus. Atlas levels are per Franklin and Paxinos, 2001. Full size image These results demonstrate that activation of Ox input to the VLPO produces rapid arousal from both NREM and REM sleep, and in a frequency-dependent manner. The arousals induced by photostimulation were typically brief. We also found that stimulation during NREM sleep, as compared with stimulations in REM sleep, doubled the length of the evoked arousals (Supplementary Fig. 1 ). Hence while activation of Ox terminals in the VLPO can evoke immediate arousal from NREM or REM sleep, only stimulation during NREM sleep was associated with longer-term effects, including an immediate post-activation suppression of sleep propensity. This finding might suggest that Ox input has downstream effects on separate NREM and REM sleep regulatory components, but these could both be located within the VLPO itself. This is consistent with previous pharmacological work showing that injections of Ox directly into the VLPO produces arousal by reducing both NREM and REM sleep and also confirming that Ox has local effects in the VLPO [11] . Effects of orexin on the cellular VLPO neurons Hence, we next studied the effects of orexin-A (Ox-A) in VLPO neurons in brain slices of WT mice (Fig. 2a–c ). We found a dual and opposite effect of Ox-A on VLPO neurons. Ox-A (0.3-1 µM) excited 35% of the neurons in the VLPO (firing frequency: +173.29 ± 41.29%; n = 21; resting membrane potential: +2.80 ± 0.44 mV; n = 26; Fig. 2d ), but unexpectedly inhibited 60% of the VLPO neurons (firing frequency: −84.37 ± 4.66%; n = 37; resting membrane potential: −4.53 ± 0.47 mV; n = 44; Fig. 2e ). Ox-A had no effects on the remaining 5% of neurons tested. We also found that while the Ox-A mediated inhibition was blocked by tetrodotoxin (TTX) or bicuculline, neither compound had an effect on Ox-A mediated excitation (Supplementary Fig. 2 ). These results demonstrate that while Ox directly excites some VLPO neurons, Ox also inhibits other VLPO neurons, but this inhibition must occur indirectly and, we predict, involves synaptic GABA signaling. We also found that the VLPO neurons that were excited by Ox-A were also excited by the cholinergic agonist carbachol and that the VLPO neurons that were inhibited by Ox-A were, instead, inhibited by carbachol (Supplementary Fig. 3). These findings suggest that the VLPO contains at least two distinct neuronal populations that respond in opposite manners to wake- promoting signals, suggesting that these two subpopulations differentially regulate sleep and arousal. Fig. 2: Dual response of orexin in VLPO. a Whole-cell recordings of VLPO neurons and post-hoc labeling of a biocytin-filled neuron (scale bars: 500 and 20 µm). b Map of the recorded neurons in VLPO ( n = 29; scale bar: 500 µm). c Most of VLPO neurons exhibit LTS (80 out of 116). d Ox-A (0.3-1 µM) excites 35% of the VLPO neurons: it increases action potential firing frequency ( n = 21; one-way ANOVA, F (2, 60) = 30.49; p < 0.0001; CTRL vs Ox-A and Ox-A vs. Wash, adj-p < 0.0001) and depolarizes the membrane potential ( n = 26; one-way ANOVA, F (2, 75) = 49.89; p < 0.0001; CTRL vs Ox-A and Ox-A vs Wash, adj-p < 0.0001). e Ox-A inhibits 60% of the VLPO neurons: it reduces action potential firing frequency ( n = 37; one-way ANOVA , F (2, 108) = 28.56; p < 0.0001; CTRL vs Ox-A and Ox-A vs Wash, adj-p < 0.0001) and hyperpolarizes membrane potential ( n = 44; one-way ANOVA, F (2, 129) =63.18; p < 0.0001; CTRL vs Ox-A and Ox-A vs Wash, adj-p < 0.0001). **** p < 0.0001, Bonferroni’s post-hoc test. Ac, anterior commissure; 3V, 3 rd ventricle; Opt, optical chiasm. Panel d and e : data are represented as means ± SEM, n refers to the number of recorded neurons and Source Data are provided as a Source Data file. Full size image VLPO GABAergic neurons show a dual response to orexin The VLPO is largely composed of GABAergic neurons, including a subpopulation that express the peptide galanin (VLPO GABA/Gal ). VLPO GABA/Gal neurons are active during sleep and promote NREM sleep [6] , [9] , [17] . Currently, little is known about the role in sleep-wake regulation of VLPO GABAergic neurons that lack galanin (VLPO GABA ). To study these neurons, we first focused on the effects of orexin (Ox-A) on the VLPO GABA population. We recorded from fluorescently labeled VLPO GABA neurons using Vgat-IRES-Cre mice into which we had placed microinjections of AAV-DIO-TdTomato or AAV-DIO-GFP into the VLPO (Supplementary Fig. 4a,b ). Both AAVs showed selective expression of fluorescent protein in Vgat-expressing neurons (Supplementary Fig. 5 and Supplementary Table 1 ). We found that Ox-A excited 42.8% of VLPO GABA neurons (firing frequency: +225.61 ± 95.01%; n = 6 and resting membrane potential: +2.95 ± 1.06 mV; n = 6) and inhibited 50% of VLPO GABA neurons (firing frequency: −72.92 ± 14.26%; n = 7 and resting membrane potential: −3.40 ± 1.13 mV; n = 7). Ox-A was without effect on the remaining 7% of the VLPO GABA neurons. These results indicate that, within the VLPO, and similar to our initial findings, there are at least two populations of VLPO GABA neurons, one that is excited by Ox and one that is instead inhibited. Previous studies showed that the VLPO GABA/Gal sleep-promoting neurons are inhibited by noradrenaline (NA) [12] , [18] . Accordingly, we found that the VLPO GABA neurons that were inhibited by Ox-A were also inhibited by NA ( n = 12) and that they expressed Gad1, Gad2, and galanin, indicating these are the VLPO GABA/Gal neurons. In contrast, we found that VLPO GABA neurons that were excited by Ox-A were also excited by NA ( n = 24) and that they expressed Gad1, and Gad2, but not galanin, i.e., were VLPO GABA neurons (Fig. 3 and Supplementary Fig. 4 ). These results confirm and extend previous studies demonstrating that the VLPO contains at least two subgroups of GABAergic neurons. The first of these subgroups, we predict, are VLPO GABA/Gal neurons, which express galanin, are inhibited by wake-promoting signals such as NA and Ox, and comprise the subpopulation of VLPO neurons that promote sleep [9] , [12] , [17] . The second subgroup, VLPO GABA neurons, lack galanin, are excited by NA and Ox and, we also predict, could be responsible for Ox-mediated feedforward inhibition of VLPO GABA/Gal neurons that would drive arousal. Fig. 3: Pharmacological and molecular diversity of the VLPO GABAergic neurons. We recorded from TdTomato labeled VLPO Vgat(+) (VLPO Vgat ) neurons in Vgat-IRES-Cre mice injected into the VLPO with AAV-DIO-TdTomato . VLPO Vgat neurons ( a top; TdTomato-labelled; sample #a18; scale bar: 20 μm) that are inhibited by NA (50 μM) express galanin. Single-cell RT-PCR results from 4 VLPO neurons inhibited by NA ( b ). The VLPO Vgat neurons ( c top ; TdTomato-labelled; sample #a30; scale bar: 20 μm) that are excited by NA do not express galanin. Single-cell RT-PCR results from 5 VLPO Vgat neurons excited by NA ( d ). Gal (182 bp), Gad1 (177 bp), Gad2 (248 bp), and Gapdh (171 bp; housekeeping gene), M marker ladder, nc negative control. e scRT-sqPCR results confirming the presence of galanin mRNA in 7 VLPO Vgat neurons inhibited by NA and/or Ox-A (NA/Ox-A(−)) and the absence of galanin mRNA in 8 VLPO Vgat neurons excited by NA and/or Ox-A (NA/Ox-A(+)). Mann–Whitney unpaired one-sided t -test, Gal NA/Ox-A(−) vs Gal NA/Ox-A(+); p = 0.0002, *** p < 0.001; values normalized to the mean Gapdh . e data are represented as means ± SEM. Panels b , d , and e Source Data are provided as a Source Data file. Full size image Orexin inhibits VLPO GABA/Gal neurons by increasing GABAergic afferent input Our next experiment focused on sleep-promoting VLPO GABA/Gal neurons. We recorded from TdTomato-labelled VLPO GABA/Gal neurons in Gal-IRES-Cre mice that had received injections of AAV-DIO-TdTomato into the VLPO. TdTomato-labeled VLPO GABA/Gal neurons expressed GABAergic markers, and as predicted, they were inhibited by NA. The majority of VLPO GABA/Gal neurons exhibited low-threshold spikes (LTS) (88.5%; n = 26), and importantly, they were inhibited by Ox-A (76.5%; action potential frequency: −84.40 ± 6.05%; n = 12; and membrane potential: −4.60 ± 0.93 mV; n = 13; Supplementary Fig. 6 ). Given again that Ox is an excitatory peptide, the finding that Ox-A inhibits VLPO neurons suggests that the observed inhibition by Ox-A must be an indirect effect and, moreover, might imply at least one additional synaptic relay and possibly the involvement of synaptic GABA. We, therefore, tested the effects of Ox-A on GABAergic synaptic input to VLPO GABA/Gal neurons. Ox-A increased the frequency of spontaneous inhibitory postsynaptic currents (sIPSCs) in 75% of the VLPO GABA/Gal neurons (+58.76 ± 13.29%; n = 9), indicating that Ox likely inhibits VLPO GABA/Gal neurons by increasing the GABAergic afferent input (Supplementary Fig. 7 ). Orexin mediates feedforward inhibition of VLPO GABA/Gal neurons via VLPO GABA neurons Given that most VLPO GABA neurons are directly excited by Ox, we next sought to determine whether VLPO GABA neurons could mediate feedforward inhibition of VLPO GABA/Gal neurons. We first tested whether VLPO GABA neurons inhibit VLPO GABA/Gal neurons (VLPO GABA → VLPO GABA/Gal input) and then whether this input was positively regulated by Ox (Fig. 4 ). Using an intersectional approach, we placed microinjections of Flp-dependent AAV-fDIO-ChR2-eYFP and Cre-dependent AAV-DIO-TdTomato into the VLPO of Vgat-Flp::Gal-IRES-Cre mice. This approach produced expression of ChR2 in VLPO neurons that express the vesicular GABA transporter (Vgat; VLPO Vgat ) and TdTomato in VLPO neurons that express galanin. RNA scope in situ hybridization confirmed selective expression of YFP and TdTomato in VLPO Vgat and VLPO GABA/Gal neurons, respectively ( Supplementary Fig. 8 and Supplementary Table 1 ). Histological assessment of the AAV injections further confirmed that ChR2 expression was restricted to the VLPO region (Fig. 4b ). We recorded from the fluorescently labeled VLPO GABA/Gal neurons at the reversal potential of the ChR2-mediated current [19] , [20] while photostimulating VLPO Vgat neurons. Photostimulation of the VLPO Vgat neurons produced short-latency opto-evoked IPSCs (oIPSCs) in VLPO GABA/Gal neurons (Fig. 4 ). Fig. 4: Orexin enhances the VLPO GABA →VLPO GABA/Gal circuit. a To study the VLPO Vgat →VLPO GABA/Gal input, we injected a mix of AAV-fDIO-ChR2-eYFP and AAV-DIO-TdTomato into the VLPO of Vgat-Flp::Gal-IRES-Cre mice ( n = 10) and recorded from TdTomato-labeled VLPO GABA/Gal neurons. To study the VLPO GABA/Gal →VLPO GABA/Gal input, we injected AAV-DIO-ChR2-mCherry into the VLPO of Gal-IRES-Cre mice ( n = 2) and recorded from mCherry-labeled VLPO GABA/Gal neurons. VLPO GABA neurons labelled in green (white arrow) and VLPO GABA/Gal neurons double-labeled in green and red (magenta arrow; scale bar: 20 µm). b Restricted transduction of AAV-fDIO-ChR2-eYFP in the VLPO of Vgat-Flp::Gal-IRES-Cre mice (YFP immunolabeling in green, scale bar: 500 μm). Injection sites from 12 mice used for in vitro CRACM recordings. c Raster plots of IPSCs in VLPO GABA/Gal neurons with photostimulation of VLPO Vgat →VLPO GABA/Gal input ( left ) and VLPO GABA/Gal →VLPO GABA/Gal input ( right; bin duration: 50 ms). d IPSC probability in response to photostimulation of the VLPO Vgat →VLPO GABA/Gal input ( black ; n = 8) and the VLPO GABA/Gal →VLPO GABA/Gal input ( grey ; n = 6; means ± SEM). Photostimulation of VLPO Vgat neurons evokes GABA A -mediated oIPSCs in VLPO GABA/Gal neurons ( e ; BIC 20 µM). Mean oIPSC amplitude and latency ( f ; n = 8; in red: means ± SEM). g Opto-evoked IPSCs recorded in TTX (1 µM + 4-AP 25–50 µM, n = 43; in red: mean ± SEM). h Ox-A (1 µM) increases oIPSC amplitude (recordings in TTX + 4-AP). i Mean oIPSC amplitude in CTRL, Ox-A and Wash ( n = 9, one-way ANOVA), F (2, 24) = 19.42, p < 0.0001, CTRL vs Ox-A and Ox-A vs Wash adj- p- value = 0.0002; means ± SEM). j Peak-scaled non-stationary fluctuation analysis showing the current/variance relationship for oIPSCs (left; control: N = 84.2, i = 0.84 pA and Ox-A: N = 139.6, i = 0.82 pA). Ox-A increases the numbers of activated GABA A channels ( center ; n = 8, CTRL vs Ox-A , p = 0.0091, p aired one-sided t -test; ** p < 0.01) without affecting the GABA A unitary current ( right ; n = 8, CTRL vs Ox-A , p = 0.2052, paired one-sided t -test; means ± SEM). Recordings at reversal potential of the ChR2-mediated current (Vh = −5 to −15 mV). Blue-light pulses (10 ms; blue bars). *** p < 0.001 Bonferroni’s post-hoc test. In grey: 30 individual oIPSCs; in black: average oIPSC. Opt, optical chiasm; 3V, 3 rd ventricle; Atlas levels are per Franklin and Paxinos, 2001. For panels d – j : n refers to the number of recorded neurons. Panels c , d , f , g , and i , j : Source Data are provided as a Source Data file. Full size image As both VLPO GABA and VLPO GABA/Gal neurons express Vgat we then tested whether collateral projections from VLPO GABA/Gal neurons (VLPO GABA/Gal → VLPO GABA/Gal ) could contribute to the oIPSCs evoked in the VLPO GABA/Gal neurons when photostimulating the VLPO GABA neurons. To explore this possibility, we placed injections of AAV-DIO-ChR2-mCherry into the VLPO of Gal-IRES-Cre mice and recorded from mCherry-labeled VLPO GABA/Gal neurons. While photostimulation of VLPO Vgat input triggered oIPSCs in 92.7% ( n = 55) of VLPO GABA/Gal neurons, photostimulation of VLPO GABA/Gal input failed to produce oIPSCs in any of the VLPO GABA/Gal neurons tested ( n = 6; Fig. 4c,d ). These results demonstrate an absence of reciprocal connectivity between VLPO GABA/Gal neurons, and more importantly show that activation of VLPO Vgat neurons by Ox is the mechanism by which the VLPO GABA → VLPO GABA/Gal circuit is activated. Photostimulation of VLPO GABA neurons produced GABA A -mediated oIPSCs in VLPO GABA/Gal neurons ( n = 8; Fig. 4e,f ). Furthermore, the oIPSCs persisted in the presence of TTX (1 µM + 4-aminopyridine, 4-AP 25–50 µM) indicating monosynaptic connectivity ( n = 43; Fig. 4g ). Ox-A increased the amplitude of oIPSCs recorded in TTX (+59.71 ± 26.3%) in 56% of VLPO GABA/Gal neurons ( n = 16; Fig. 4h,i ) indicating a presynaptic effect. All together these results demonstrate that VLPO GABA/Gal neurons can be inhibited by local VLPO GABA neurons, and that activity of this circuit is enhanced by Ox. We next applied peak-scaled non-stationary fluctuation analysis [21] , [22] , [23] to assess whether Ox-A enhances the VLPO GABA → VLPO GABA/Gal input by increasing the unitary GABA A current or the number of activated GABA A receptors or both. For each cell, we obtained parabolic variance vs current amplitude curves. We estimated the ionic channel current ( i ) and the number of activated channels ( N ) open at the peak of the oIPSCs, in control and during Ox-A application. We found that Ox-A increased the oIPSC amplitude by enhancing the number of activated GABA A channels (+89.33 ± 33.23 %; n = 8, p = 0.0091, paired t -test) without affecting the GABA A unitary current (Fig. 4j ). These results are a strong indication that Ox enhances the VLPO GABA → VLPO GABA/Gal input by increasing the amount of GABA being released. VLPO GABA/Gal and VLPO GABA neurons have distinct molecular profiles and expression of orexin receptors is restricted to a subset of VLPO GABA neurons To characterize the transcriptional profile of the VLPO GABA/Gal and VLPO GABA neurons, we retrieved and clustered the publicly available data of the preoptic area (POA) previously reported by Moffitt and colleagues in 2018 [24] . Our bioinformatic analysis confirmed their earlier published POA clusters along with the cellular markers (Supplementary Fig. 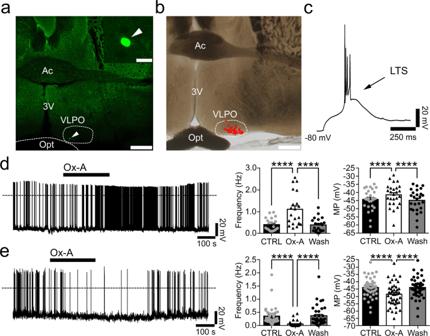Fig. 2: Dual response of orexin in VLPO. aWhole-cell recordings of VLPO neurons andpost-hoclabeling of a biocytin-filled neuron (scale bars: 500 and 20 µm).bMap of the recorded neurons in VLPO (n= 29; scale bar: 500 µm).cMost of VLPO neurons exhibit LTS (80 out of 116).dOx-A (0.3-1 µM) excites 35% of the VLPO neurons: it increases action potential firing frequency (n= 21; one-way ANOVA,F(2, 60)= 30.49;p< 0.0001; CTRL vs Ox-A and Ox-A vs. Wash,adj-p< 0.0001) and depolarizes the membrane potential (n= 26; one-way ANOVA,F(2, 75)= 49.89;p< 0.0001; CTRL vs Ox-A and Ox-A vs Wash,adj-p< 0.0001).eOx-A inhibits 60% of the VLPO neurons: it reduces action potential firing frequency (n= 37; one-way ANOVA, F(2, 108)= 28.56;p< 0.0001; CTRL vs Ox-A and Ox-A vs Wash,adj-p< 0.0001) and hyperpolarizes membrane potential (n= 44; one-way ANOVA,F(2, 129)=63.18;p< 0.0001; CTRL vs Ox-A and Ox-A vs Wash,adj-p< 0.0001). ****p< 0.0001, Bonferroni’spost-hoctest. Ac, anterior commissure; 3V, 3rdventricle; Opt, optical chiasm. Paneldande: data are represented as means ± SEM,nrefers to the number of recorded neurons and Source Data are provided as a Source Data file. 9 , Supplementary Table 2 ). Using the spatial transcriptomic ( Multiplexed Error Robust Fluorescence In Situ Hybridization : MERFISH) data provided in the same study, we isolated the neuronal clusters of the VLPO region and generated a VLPO atlas of 4174 neurons x 21,043 genes divided into 20 (#0-19) clusters (Supplementary Fig. 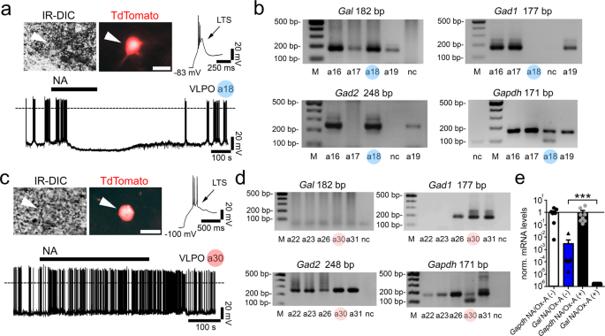Fig. 3: Pharmacological and molecular diversity of the VLPO GABAergic neurons. We recorded from TdTomato labeled VLPO Vgat(+) (VLPOVgat) neurons inVgat-IRES-Cremice injected into the VLPO withAAV-DIO-TdTomato. VLPOVgatneurons (atop;TdTomato-labelled; sample #a18; scale bar: 20 μm) that are inhibited by NA (50 μM) express galanin. Single-cell RT-PCR results from 4 VLPO neurons inhibited by NA (b). The VLPOVgatneurons (ctop; TdTomato-labelled; sample #a30; scale bar: 20 μm) that are excited by NA do not express galanin. Single-cell RT-PCR results from 5 VLPOVgatneurons excited by NA (d). Gal(182 bp),Gad1(177 bp),Gad2(248 bp), andGapdh(171 bp; housekeeping gene), M marker ladder, nc negative control.escRT-sqPCR results confirming the presence ofgalaninmRNA in 7 VLPOVgatneurons inhibited by NA and/or Ox-A (NA/Ox-A(−)) and the absence ofgalaninmRNA in 8 VLPOVgatneurons excited by NA and/or Ox-A (NA/Ox-A(+)). Mann–Whitney unpaired one-sidedt-test,GalNA/Ox-A(−) vsGalNA/Ox-A(+);p= 0.0002, ***p< 0.001; values normalized to the meanGapdh.edata are represented as means ± SEM. Panelsb,d, andeSource Data are provided as a Source Data file. 10 , 11 , Supplementary Table 3 ). We then compared the molecular identity of GABAergic neuronal groups in VLPO that either express or lack expression of galanin, by performing differential gene expression. The VLPO GABA/Gal and VLPO GABA groups comprised 3 clusters (515 neurons) and 12 clusters (2,911 neurons), respectively. We found that the VLPO GABA/Gal and VLPO GABA groups have very distinct transcriptional profiles (Fig. 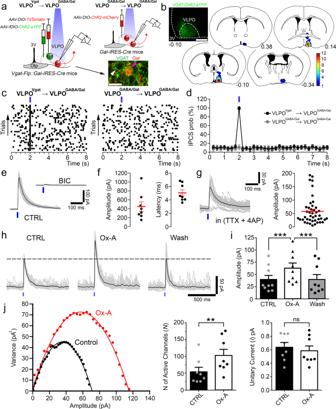Fig. 4: Orexin enhances the VLPOGABA→VLPOGABA/Galcircuit. aTo study the VLPOVgat→VLPOGABA/Galinput, we injected a mix ofAAV-fDIO-ChR2-eYFPandAAV-DIO-TdTomatointo the VLPO ofVgat-Flp::Gal-IRES-Cremice (n= 10) and recorded from TdTomato-labeled VLPOGABA/Galneurons. To study the VLPOGABA/Gal→VLPOGABA/Galinput, we injectedAAV-DIO-ChR2-mCherryinto the VLPO ofGal-IRES-Cremice (n= 2) and recorded from mCherry-labeled VLPOGABA/Galneurons. VLPOGABAneurons labelled in green (white arrow) and VLPOGABA/Galneurons double-labeled in green and red (magenta arrow; scale bar: 20 µm).bRestricted transduction ofAAV-fDIO-ChR2-eYFPin the VLPO ofVgat-Flp::Gal-IRES-Cremice (YFP immunolabeling in green, scale bar: 500 μm). Injection sites from 12 mice used for in vitro CRACM recordings.cRaster plots of IPSCs in VLPOGABA/Galneurons with photostimulation of VLPOVgat→VLPOGABA/Galinput (left) and VLPOGABA/Gal→VLPOGABA/Galinput (right;bin duration: 50 ms).dIPSC probability in response to photostimulation of the VLPOVgat→VLPOGABA/Galinput (black;n= 8) and the VLPOGABA/Gal→VLPOGABA/Galinput (grey;n= 6; means ± SEM). Photostimulation of VLPOVgatneurons evokes GABAA-mediated oIPSCs in VLPOGABA/Galneurons (e;BIC 20 µM). Mean oIPSC amplitude and latency (f; n= 8; in red: means ± SEM).gOpto-evoked IPSCs recorded in TTX (1 µM + 4-AP 25–50 µM,n= 43; in red: mean ± SEM).hOx-A (1 µM) increases oIPSC amplitude (recordings in TTX + 4-AP).iMean oIPSC amplitude in CTRL, Ox-A and Wash (n= 9, one-way ANOVA),F(2, 24)= 19.42,p< 0.0001, CTRL vs Ox-A and Ox-A vs Wash adj-p-value = 0.0002; means ± SEM).jPeak-scaled non-stationary fluctuation analysis showing the current/variance relationship for oIPSCs (left; control:N= 84.2,i= 0.84 pA and Ox-A:N= 139.6,i= 0.82 pA). Ox-A increases the numbers of activated GABAAchannels (center;n= 8, CTRL vs Ox-A, p= 0.0091,paired one-sidedt-test; **p< 0.01) without affecting the GABAAunitary current (right;n= 8, CTRL vs Ox-A, p= 0.2052, paired one-sidedt-test; means ± SEM). Recordings at reversal potential of the ChR2-mediated current (Vh = −5 to −15 mV). Blue-light pulses (10 ms; blue bars). ***p< 0.001 Bonferroni’spost-hoctest. In grey: 30 individual oIPSCs; in black: average oIPSC. Opt, optical chiasm; 3V, 3rdventricle; Atlas levels are per Franklin and Paxinos, 2001. For panelsd–j:nrefers to the number of recorded neurons. Panelsc,d,f,g, andi,j: Source Data are provided as a Source Data file. 5a-b and Supplementary Table 4 ), but also share commonalities. For example, both cell populations expressed markers for GABA synthesis and transmission ( Slc32a1 , Gad1 , Gad2 ) and neither expressed the Vglut2 gene ( Slc17a6 ). In agreement with our electrophysiology data, orexin/hypocretin receptors (Hcrtrs) were not expressed in any of the three VLPO GABA/Gal clusters, whereas cluster #1 of the VLPO GABA group (Fig. 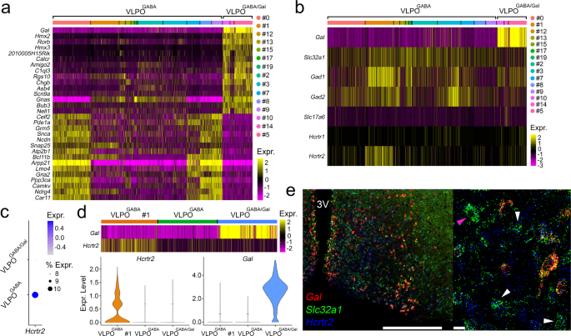Fig. 5: Differential expression profiles and orexin receptor expression in VLPOGABA/Galand VLPOGABAneurons. Heat maps representing the expression levels of the top 30 differentially expressed genes ranked byadj-p(panela; top 15 hypo- and top 15 hyper-expressed) and expression levels of GABAergic genes (Slc32a1,Gad1,Gad2),Hcrtr1, Hcrtr2,GalandSlc17a6(panelb) in the VLPOGABA(#0–3; 7–9; 12, 13, 15, 17, 19) and VLPOGABA/Gal(#5, 10, 14) clusters.Hcrtr2positive neurons were largely restricted to VLPOGABAcluster #1.cDot plot representing the average expression ofHcrtr2gene (x axis) in VLPOGABAand VLPOGABA/Galgroups (y axis). Dot size: percentage of neurons that expresses a specific gene (bottom right). Color intensity: expression level (top right).dHeat map ofGalandHcrtr2gene expression levels in VLPOGABAcluster #1 (orange; 489 neurons), in all the other VLPOGABAclusters (#0, 2, 3; 7–9; 12, 13, 15, 17, 19; green; down sampled to 515 neurons) and merged VLPOGABA/Galclusters (#5, 10, 14; cyan; 515 neurons). Violin plots forHcrtr2(bottom left) andGal(bottom right) differential gene expression: VLPOGABAcluster #1 (orange), all the other VLPOGABAclusters (#0, 2, 3; 7–9; 12, 13, 15, 17, 19; green) and VLPOGABA/Galclusters (#5, 10, 14; cyan).Hcrtr2is expressed in VLPOGABA#1 (VLPOGABA#1 vs VLPOGABA/Galadj-pvalue = 4.98E−32; VLPOGABA#1 vs. VLPOGABA(#0, 2, 3; 7–9; 12, 13, 15, 17, 19) adj-pvalue = 1.63E−114).Galis expressed in VLPOGABA/Galneurons (VLPOGABA#1 vs VLPOGABA/Galadj-pvalue = 1.26E−144; VLPOGABA(#0, 2, 3; 7–9; 12, 13, 15, 17, 19) vs VLPOGABA/Galadj-pvalue = 0). Heat map and Dot plot expression values are represented as z-scores. Expression levels is color- coded in the legend. In the heat maps,x-axis: individual clusters color-coded bar;y-axis: genes. As color dots: Cluster IDs (right). Test used:Wilcoxon Rank Sum two-sidedBonferroni-corrected Test.eExpression in VLPO ofGal(red),Slc32a1(green) andHcrtr2(pseudo colored in blue) mRNAs. White arrows:Slc32a1(+),Hcrtr2(+) andGal(−) neurons; magenta arrows:Slc32a1(+),Hcrtr2(−) andGal(−) neurons. Scale bars: 500 and 20 µm (bottom right). 3V, 3rdventricle. Source Data are provided as a Source Data file. 5c,d and Supplementary Table 5 ), which is the second-largest cluster of the VLPO GABA groups, expressed Hcrtr2 RNA (Ox2R) (489 neurons; Supplementary Tables 6, 7 ). Hcrtr1 RNA (Ox1R) was not detected in any of the VLPO clusters, as previously reported by in situ hybridization [25] (Fig. 5b ). Fig. 5: Differential expression profiles and orexin receptor expression in VLPO GABA/Gal and VLPO GABA neurons. Heat maps representing the expression levels of the top 30 differentially expressed genes ranked by adj-p (panel a ; top 15 hypo- and top 15 hyper-expressed) and expression levels of GABAergic genes ( Slc32a1 , Gad1 , Gad2 ), Hcrtr1, Hcrtr2 , Gal and Slc17a6 (panel b ) in the VLPO GABA (#0–3; 7–9; 12, 13, 15, 17, 19) and VLPO GABA/Gal (#5, 10, 14) clusters. Hcrtr2 positive neurons were largely restricted to VLPO GABA cluster #1. c Dot plot representing the average expression of Hcrtr2 gene ( x axis ) in VLPO GABA and VLPO GABA/Gal groups ( y axis ). Dot size: percentage of neurons that expresses a specific gene ( bottom right ). Color intensity: expression level ( top right ). d Heat map of Gal and Hcrtr2 gene expression levels in VLPO GABA cluster #1 (orange; 489 neurons), in all the other VLPO GABA clusters (#0, 2, 3; 7–9; 12, 13, 15, 17, 19; green; down sampled to 515 neurons) and merged VLPO GABA/Gal clusters (#5, 10, 14; cyan; 515 neurons). Violin plots for Hcrtr2 ( bottom left ) and Gal ( bottom right ) differential gene expression: VLPO GABA cluster #1 (orange), all the other VLPO GABA clusters (#0, 2, 3; 7–9; 12, 13, 15, 17, 19; green) and VLPO GABA/Gal clusters (#5, 10, 14; cyan). Hcrtr2 is expressed in VLPO GABA #1 (VLPO GABA #1 vs VLPO GABA/Gal adj- p value = 4.98E−32; VLPO GABA #1 vs. VLPO GABA (#0, 2, 3; 7–9; 12, 13, 15, 17, 19) adj- p value = 1.63E−114). Gal is expressed in VLPO GABA/Gal neurons (VLPO GABA #1 vs VLPO GABA/Gal adj- p value = 1.26E−144; VLPO GABA (#0, 2, 3; 7–9; 12, 13, 15, 17, 19) vs VLPO GABA/Gal adj- p value = 0). Heat map and Dot plot expression values are represented as z-scores. Expression levels is color- coded in the legend. In the heat maps, x-axis : individual clusters color-coded bar; y-axis : genes. As color dots: Cluster IDs ( right ). Test used: Wilcoxon Rank Sum two-sided Bonferroni-corrected Test. e Expression in VLPO of Gal (red), Slc32a1 (green) and Hcrtr2 (pseudo colored in blue) mRNAs. White arrows: Slc32a1 (+), Hcrtr2 (+) and Gal (−) neurons; magenta arrows: Slc32a1 (+), Hcrtr2 (−) and Gal (−) neurons. Scale bars: 500 and 20 µm ( bottom right ). 3V, 3 rd ventricle. Source Data are provided as a Source Data file. Full size image We confirmed these bioinformatic results using RNA scope in situ hybridization. Our in situ analysis confirmed an absence of expression of Hcrtr2 mRNA in VLPO neurons that expressed both Slc32a1 ( Vgat) and Gal mRNAs (i.e., VLPO GABA/Gal ). In addition, Hcrtr2 mRNA was expressed in 28.5% of VLPO neurons that express Slc32a1 but not Gal mRNAs (i.e., VLPO GABA ) (Fig. 5e ; Supplementary Table 8 ) . These results confirm our in vitro recording findings that only VLPO GABA neurons, or a subset thereof, are capable of responding directly to Ox and hence represent a likely ‘gateway’ for Ox signaling into the cellular VLPO network. Inputs from orexin neurons excite VLPO GABA neurons We next verified functional synaptic connectivity between Ox and VLPO neurons using in vitro CRACM recordings. We expressed ChR2 in Ox neurons by injecting AAV-DIO-ChR2-eYFP or AAV-DIO-ChR2-mCherry into the lateral hypothalamus of Ox-IRES-Cre mice. We then recorded from VLPO neurons in brain slices while photostimulating the Ox axon terminals (Fig. 6a ). We confirmed selective expression of YFP or mCherry in Ox neurons by immunolabeling (Fig. 1d and Supplementary Table 1 ). Histological assessment of the AAV injections confirmed that expression of ChR2 was restricted to the Ox field (Fig. 6b ). Photostimulation of the Ox → VLPO input produced opto-evoked excitatory postsynaptic currents (oEPSCs) in 24% of recorded VLPO neurons ( n = 63). DNQX (20–200 µM; n = 4) abolished the oEPSCs, indicating release of glutamate and AMPA-mediated signaling in VLPO neurons (Fig. 6c–e ). Neurons that responded to photostimulations with glutamate-mediated oEPSCs displayed no changes in holding currents nor in resting membrane potentials during or after 60 s-long photostimulation trains indicating no detectable release of Ox (Fig. 6f ). Fig. 6: Orexin input excites VLPO GABA neurons by glutamate release (Ox → VLPO GABA ). a AAV-DIO-ChR2-eYFP injected into the Ox field of Ox-IRES-Cre mice and recordings from VLPO neurons. b Injection sites of 15 Ox-IRES-Cre mice used for in vitro CRACM ( n = 10 mice) and in vivo optogenetics ( n = 5 mice). c Photostimulation of Ox → VLPO input evokes AMPA-mediated oEPSCs in VLPO neurons (DNQX 200 µM; in grey: 30 individual oEPSCs; in black: average oEPSC). d Raster plot of EPSCs in a VLPO neuron before, during, and after photostimulation of the Ox → VLPO input (50 ms bins). e Average EPSC probability of VLPO neurons that responded ( n = 13; black) and did not respond ( n = 48; grey; means ± SEM) to the photostimulation of Ox input. f No changes in holding currents in response to photostimulation trains (60 s at 10 and 20 Hz; 10 ms light pulses) in neurons activated by the Ox → VLPO input with glutamate-mediated oEPSCs. The VLPO GABA neurons are activated by the Ox → VLPO input. The VLPO neurons that responded to photostimulation of the Ox → VLPO input ( n = 7) are excited by NA ( g ) and/or do not express galanin mRNA ( h ; scRT-sqPCR). Specifically 4 neurons were tested for both the responses to NA and for the presence of Gal mRNA, 2 only for NA, and 1 only for Gal mRNA. Mean effects of NA on the action potential frequency ( g left ; paired one-sided t -test, CTRL vs NA, p = 0.0033; n = 4) and membrane potential ( g, right; paired one-sided t -test, CTRL vs NA, p = 0.0017; n = 6). Results from scRT-sqPCR for Gapdh and galanin ( Gal ) from 5 VLPO neurons Ox → VLPO input connected (conn) are compared to 13 controls (ctrl) VLPO GABA/Gal neurons ( h ; ctrl: sampled from recorded VLPO GABA/Gal TdTomato-labeled neurons from Gal-IRES-Cre mice injected with AAV-DIO-TdTomato ). Mann-Whitney unpaired one-sided t -test, Gal (conn) vs Gal (ctrl); p = 0.0001. Values are normalized to the mean Gapdh . Means ± SEM. i oEPSC amplitude ( left ) and latency ( right ) in 15 VLPO neurons (blue dots: identified VLPO GABA neurons; in red: means ± SEM). Recordings at V h = −70 mV; 10 ms blue-light pulses (blue bars). *** p < 0.001 and ** p < 0.01. 3V 3 rd ventricle, Opt optical chiasm, f fornix, mt mammillothalamic tract, LH lateral hypothalamus. Atlas levels are per Franklin and Paxinos, 2001. For panels e and g : n refers to the number of recorded neurons. Panel d–e and g–i: Source Data file. Full size image To identify the postsynaptic target neurons in VLPO of this Ox input, we tested the VLPO neurons that responded to photostimulation for their response to NA and/or for expression of Gal by scRT-sqPCR ( n = 7). We found that 6 of the recorded neurons were excited by NA (Fig. 6g ) whereas 1 was inhibited. All VLPO neurons that responded to photostimulation of the Ox → VLPO input lacked Gal mRNA (Fig. 6h ). Altogether, these results demonstrate that Ox nerve terminals exclusively contact and activate VLPO GABA neurons (Fig. 7 ). Fig. 7: Orexin neurons promote wakefulness by inhibiting sleep-promoting VLPO GABA/Gal neurons via feed-forward inhibition. Orexin neurons promote arousal through their projections to the VLPO. Orexin input to the VLPO directly activates VLPO GABAergic neurons that do not express galanin (VLPO GABA ) via co-release of Ox and glutamate. In turn, VLPO GABA neurons inhibit VLPO GABA/Gal sleep-promoting neurons to produce wakefulness. Full size image Here we demonstrate the existence of a functional polysynaptic circuit between the Ox neurons and sleep-promoting VLPO GABA/Gal neurons. We further demonstrate that selective activation of the Ox → VLPO GABA → VLPO GABA/Gal circuit is potently wake-promoting in vivo. And our in vitro results demonstrate that Ox directly activates Hcrtr2-expressing VLPO GABA neurons, but not VLPO GABA/Gal neurons. These results identify a clearly delineated polysynaptic circuit by which Ox neurons can effectively “turn off” sleep-promoting VLPO GABA/Gal neurons to promote arousal in vivo. Our findings specifically support a circuit model in which the Ox input (and co-released glutamate) exerts its excitatory influence on VLPO GABA interneurons, including in the case of Hcrtr2-expressing VLPO GABA interneurons, which in turn inhibit sleep-promoting VLPO GABA/Gal neurons to promote and stabilize wakefulness. In this verified circuit model, loss of Ox, as occurs in narcolepsy, would result in a reduction in excitatory tone on VLPO GABA neurons, thereby reducing feedforward inhibition of VLPO GABA/Gal neurons and biasing their sustained activity and, hence, the sleep state. A reciprocal inhibitory relationship between the VLPO and components of the brain’s arousal system, including hypothalamic Ox neurons [26] , [27] , is thought to support both the consolidation of behavioral state and the ability to rapidly and completely transition between behavioral states, e.g., wake to sleep [28] . This circuit arrangement has been conceptualized as being analogous to an electronic flip-flop switch, which possesses the desirable properties of being both self-stabilizing and highly stable in their ‘on’ or ‘off’ states. Hence, under normal neurobiological conditions, this flip-flop circuit arrangement ensures strong state boundary control, i.e., unstable intermediate states are avoided. However, when this circuitry is damaged, as occurs in various parasomnias and sleep-wake disorders such as narcolepsy, the ‘weakened’ switch operates closer to the boundary zone, leading to a greater percentage of time spent in unstable transition or intermediate states. In the case of narcolepsy, these frequent and unwanted transitions into the boundary zone result in the manifestation of debilitating physical symptoms including fragmentation of sleep or wake, cataplexy, sleep paralysis, hallucinations, and sleep-onset rapid-eye-movement sleep events (SOREMs). A similar phenomenon occurs during aging, when cell loss in the VLPO leads to weakening of the “sleep side” of the switch, in turn resulting in sleep fragmentation and daytime napping, both of which are frequent complaints in the elderly [29] , [30] . During wakefulness, sleep-promoting VLPO GABA/Gal neurons are inhibited by afferent inputs from many sources [16] , including the Ox neurons. Intermingled however with VLPO GABA/Gal neurons are additional GABAergic neurons (VLPO GABA ) that lack galanin and appear to be active during wakefulness [12] , [18] , [31] , [32] , [33] . In this regard, they are similar to the GABA neurons in the more caudal lateral hypothalamus that also promote wakefulness by inhibiting the VLPO GABA/Gal neurons [13] . Here, we show that Ox directly excites a subset of Hcrtr2-expressing VLPO GABA neurons, and in turn through their local collaterals, these neurons inhibit the sleep-promoting VLPO GABA/Gal cell population. Findings from the present study, therefore, support a circuit model in which local VLPO GABA neurons function as an interface between afferent inputs to the VLPO and sleep-promoting VLPO GABA/Gal neurons. In other words, Ox, and possibly other wake-promoting signals, via feedforward inhibition, inhibit VLPO GABA/Gal neurons to produce arousal, and sleep-promoting signals, in turn via disinhibition, activate VLPO GABA/Gal neurons to produce sleep. This intra-VLPO circuit mechanism for promoting state transitions could be shared by most, if not all, wake- and sleep-promoting afferences that modulate VLPO activity [32] , [34] , [35] , [36] , [37] . Our model further predicts that VLPO GABA neurons are wake-active and, possibly, wake-promoting. In fact, recordings in the VLPO have uncovered neurons that are active in wakefulness [8] , [33] and optogenetic activation of Gad2-expressing VLPO neurons [which likely activates both VLPO GABA/Gal and VLPO GABA neurons] produces arousal, suggesting that co-activation of VLPO GABA and VLPO GABA/Gal neurons can override the ability of VLPO GABA/Gal neurons to produce sleep [38] . 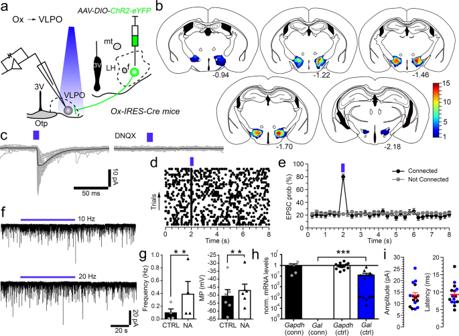Fig. 6: Orexin input excites VLPOGABAneurons by glutamate release (Ox → VLPOGABA). aAAV-DIO-ChR2-eYFPinjected into the Ox field ofOx-IRES-Cremice and recordings from VLPO neurons.bInjection sites of 15Ox-IRES-Cremice used for in vitro CRACM (n= 10 mice) and in vivo optogenetics (n= 5 mice).cPhotostimulation of Ox → VLPO input evokes AMPA-mediated oEPSCs in VLPO neurons (DNQX 200 µM; in grey: 30 individual oEPSCs; in black: average oEPSC).dRaster plot of EPSCs in a VLPO neuron before, during, and after photostimulation of the Ox → VLPO input (50 ms bins).eAverage EPSC probability of VLPO neurons that responded (n= 13; black) and did not respond (n= 48; grey; means ± SEM) to the photostimulation of Ox input.fNo changes in holding currents in response to photostimulation trains (60 s at 10 and 20 Hz; 10 ms light pulses) in neurons activated by the Ox → VLPO input with glutamate-mediated oEPSCs. The VLPOGABAneurons are activated by the Ox → VLPO input. The VLPO neurons that responded to photostimulation of the Ox → VLPO input (n= 7) are excited by NA (g) and/or do not expressgalaninmRNA (h; scRT-sqPCR). Specifically 4 neurons were tested for both the responses to NA and for the presence ofGalmRNA, 2 only for NA, and 1 only forGalmRNA. Mean effects of NA on the action potential frequency (gleft; paired one-sidedt-test, CTRL vs NA,p= 0.0033;n= 4) and membrane potential (g, right;paired one-sidedt-test, CTRL vs NA,p= 0.0017;n= 6). Results from scRT-sqPCR forGapdhandgalanin(Gal) from 5 VLPO neurons Ox → VLPO input connected (conn) are compared to 13 controls (ctrl) VLPOGABA/Galneurons (h;ctrl: sampled from recorded VLPOGABA/GalTdTomato-labeled neurons fromGal-IRES-Cremice injected withAAV-DIO-TdTomato). Mann-Whitney unpaired one-sidedt-test,Gal(conn) vsGal(ctrl);p= 0.0001. Values are normalized to the meanGapdh. Means ± SEM.ioEPSC amplitude (left) and latency (right) in 15 VLPO neurons (blue dots: identified VLPOGABAneurons; in red: means ± SEM). Recordings at Vh= −70 mV; 10 ms blue-light pulses (blue bars). ***p< 0.001 and **p< 0.01. 3V 3rdventricle, Opt optical chiasm, f fornix, mt mammillothalamic tract, LH lateral hypothalamus. Atlas levels are per Franklin and Paxinos, 2001. For panelseandg:nrefers to the number of recorded neurons. Panel d–e and g–i: Source Data file. 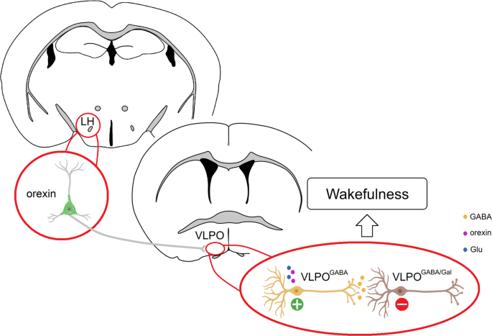Fig. 7: Orexin neurons promote wakefulness by inhibiting sleep-promoting VLPOGABA/Galneurons via feed-forward inhibition. Orexin neurons promote arousal through their projections to the VLPO. Orexin input to the VLPO directly activates VLPO GABAergic neurons that do not express galanin (VLPOGABA) via co-release of Ox and glutamate. In turn, VLPOGABAneurons inhibit VLPOGABA/Galsleep-promoting neurons to produce wakefulness. A better understanding of the synaptic, cellular, and circuit bases by which Ox neurons stabilize and maintain wakefulness has important implications for treating patients with neurological disorders associated with arousal dysfunction. For instance, patients suffering from narcolepsy exhibit debilitating sleepiness, sleep attacks, and wake- instability, which take a tremendous toll on quality of life. At present, these symptoms are largely addressed clinically through the provision of stimulants, which themselves possess unwanted side effects. We show here that Ox exerts its wake-promoting effects, at least in part, through indirect inhibition of sleep-promoting VLPO GABA/Gal neurons, and our electrophysiological and single-cell transcriptomics findings uncover and characterize two molecularly-distinct VLPO cell populations. There exists considerable redundancy in the brain’s arousal circuitry, with only a few ‘nodes’ having been established as truly necessary for arousal maintenance [39] , [40] , [41] , [42] , i.e., loss or disruption produces a chronic reduction in arousal level. Similarly, Ox neurons likely produce arousal (and contribute to state stabilization) through multiple projections [14] , wherein each post-synaptic ‘target’ of Ox neurons likely contributes to arousal control and stabilization, yet any given individual ‘target’ in isolation is unlikely necessary for arousal maintenance. Taken together, our findings suggest that VLPO GABA neurons, or a subset thereof, may represent a ‘common point of entry’ for a wide range of inputs into the intra-VLPO cellular network. These findings also suggest the possibility of new ‘targets’ for the development of more selective pharmacologic strategies for treating the crippling inability to maintain consolidated wakefulness in narcolepsy and in other neurodegenerative, neurodevelopmental, and neuropsychiatric diseases in which disordered arousal, including even hyperarousal (e.g., insomnia), is a prominent clinical feature. Animals and stereotaxic viral injections Mice were treated in accordance with guidelines from the National Institute of Health Guide for the Care and Use of Laboratory Animals . All protocols were approved by Beth Israel Deaconess Medical Center Institutional Animal Care and Use Committee and all efforts were directed to minimize the number of animals and their suffering. Mice were held at temperature of 22 ± 1 °C (40−60% of humidity) and on a 12 h light/dark cycle with available food and water access ad libitum. We used adult mice, 6-12 weeks of age, and an equal proportion of male and female mice. We used: 55 C57BL/6J (WT); 33 Vgat-IRES-Cre ; 25 Galanin-IRES-Cre ( Gal-IRES-Cre ); 11 Orexin-IRES-Cre ( Ox-IRES-Cre ) and 10 Vgat-Flp::Gal-IRES-Cre mice. WT mice were purchased from The Jackson Laboratory (Jax, Bar Harbor, ME). Vgat-IRES-Cre mice (obtained by The Jackson Laboratory: Jax Slc32a1 tm2(cre)Lowl /J, Cat. #016962) express Cre-recombinase under the control of vesicular GABA transporter ( Vgat, Slc32a1 ) gene, to restrict the recombination in GABAergic neurons [43] . The Gal-IRES-Cre mice express Cre-recombinase under the galanin ( Gal ) gene promoter [9] , [44] and were given to us by Dr. Ramalingam Vetrivelan (Neurology Department, BIDMC, Boston, MA). The Vgat-Flp::Gal-IRES-Cre mice express Flp- recombinase in Vgat expressing neurons and Cre-recombinase in galanin expressing neurons and were obtained by crossing the Slc32a1 tm1.1(flpo)Hze mice ( Vgat-Flp ; obtained by The Jackson Laboratory: Jax B6.Cg-Slc32a1 tm1.1(flpo)Hze /J, Cat. #029591) with the Gal-IRES-Cre mice. To activate the input from Ox neurons to VLPO (in vivo and in vitro recordings), we expressed ChR2-mCherry or ChR2-eYFP in the Ox neurons using two Cre-dependent AAVs: the AAV-DIO-ChR2-mCherry ( rAAV8-Ef1a-DIO-hChR2(H134R)-mCherry ; 1.5 × 10 13 virus molecules/ml; UNC Gene Therapy Center) and the AAV-DIO-ChR2-eYFP ( AAV10-Ef1a-DIO-hChR2(H134R)-eYFP ; 6.6×10 12 virus molecules/ml; provided by Dr. P.M.F.). As previously described [45] we placed two bilateral injections of AAV-DIO-ChR2-mCherry or AAV-DIO-ChR2-eYFP into the lateral hypothalamus of Ox-IRES-Cre mice (300 nl for each of the 4 injections, 2 per side: AP: −0.7 mm, DV: −5.0 mm, ML: ± 1.0 mm and AP: −1.6 mm, DV: −5.0 mm, ML: ± 0.8 mm). Animals used for the sleep studies were also instrumented for optogenetic stimulations and EEG/EMG recordings. EEG/EMG recordings started four weeks after the surgeries. Four to six weeks after the AAV injections we recorded in brain slices for in vitro CRACM recordings. To identify VLPO GABAergic and galanin neurons in recording slices we labeled them with TdTomato or GFP by placing bilateral microinjections of AAV-DIO-TdTomato ( AAV10-Ef1a-DIO-TdTomato ; was provided by Dr. P.M.F.) or AAV-DIO-GFP ( rAAV8- DIO-GFP ; 6×10 12 virus molecules/ml; prepared by the UNC Gene Therapy Center, University of North Carolina, Chapel Hill, NC) into the VLPO (180 nl; AP: 0.26 mm, DV: −5.2 mm, ML: ± 0.6 mm) of Vgat-IRES-Cre, Gal-IRES-Cre and Vgat-Flp::Gal-IRES-Cre mice. Two weeks after the AAV injections, we recorded in brain slices from fluorescently labeled Vgat or galanin expressing neurons. To study the VLPO internal circuit by in vitro CRACM recordings, we used two Cre-dependent AAVs: one AAV that codes for ChR2 ( AAV-DIO-ChR2-mCherry ) and one that codes for TdTomato ( AAV-DIO-TdTomato ). We also used a Flp-dependent AAV that codes for ChR2-eYFP, the AAV-fDIO-ChR2-eYFP ( AAVDJ-Ef1a-fDIO-ChR2-eYFP; 2 × 10 12 virus molecules/ml; UNC Gene Therapy Center). Specifically, to activate collateral inputs between VLPO galanin neurons, we unilaterally injected AAV-DIO-ChR2-mCherry (35–50 nl) into the VLPO of Gal-IRES-Cre mice (AP: 0.26 mm, DV: −5.2 mm, ML: ± 0.6 mm) and we recorded from VLPO galanin neurons. To activate the input from local VLPO GABAergic neurons to VLPO galanin neurons, we unilaterally injected the Flp-dependent AAV-fDIO-ChR2-eYFP (35-50 nl) and the Cre-dependent AAV-DIO-TdTomato (180 nl) into the VLPO of Vgat-Flp::Gal-IRES-Cre mice (AP: + 0.26 mm, DV: −5.2 mm, ML: ± 0.6 mm). This results in the expression of ChR2-eYFP in the GABAergic neurons and TdTomato in galanin neurons. We recorded from VLPO galanin neurons labeled by TdTomato. Stereotaxic coordinates for all the AAV injections were based on mouse brain atlas by Paxinos and Franklin (2001). We conducted slice recordings 4-6 weeks after the AAV injections. Generation of Ox-IRES-Cre knock-in mice These mice were generated, validated, and kindly provided by Drs. D.K., T.M., B.B.L., and T.E.S. The Ox-IRES-Cre mice express the Cre-recombinase under the control of the endogenous orexin/hypocretin ( Ox/Hcrt ) gene locus. Briefly, the generation of the gene targeting construct was performed through the help of a modified BAC clone [46] that contained the Ox/Hcrt genomic sequence, as previously reported [47] . This BAC-derived construct spans the region 5 kb upstream of the IRES site and 2 kb downstream of the Cre site inserted into 3′-end genomic region. Then, it was electroporated into mouse embryonic stem (ES) cells (W4/129S6, Taconic, Germantown, NY). Correctly targeted ES cells were identified and then injected into blastocysts to generate chimeras. The male chimeras mice were bred to mice bearing a Flp-recombinase transgene, in order to remove the selection marker neomycin. The Cre-recombinase activity was verified in the hypothalamus by crossing male chimeras to Ai14 Cre reporter line (obtained by The Jackson Laboratory: Jax B6;129S6- Gt(ROSA)26Sor tm14(CAG-tdTomato)Hze /J, Cat. #007908) [47] . EEG/EMG and optical fiber implants We used Ox-IRES-Cre ( n = 5 mice) and WT ( n = 3 mice as controls). Following bilateral injections of AAV-DIO-ChR2-mCherry into the lateral hypothalamus mice underwent a second surgery to implant a headstage for EEG and EMG recordings and optical fibers for bilateral optogenetic stimulation of the Ox input to VLPO. The headstages were custom-made in-house by assembling a 6-pin connector (Heilind Electronics, catalog #MMX853-43-006-10-001000), 4 EEG screws (Pinnacle, catalog# 8403), and 2 flexible EMG wire electrodes (Plastics One, catalog #E363). During surgery, two burr holes were drilled in the skull of the anesthetized mice immediately above the VLPO (AP = + 0.4 mm; ML = ± 0.7 mm) for placement of the optical fibers. Each optical fiber was stereotaxically guided into position (DV = −5.0 mm). We drilled 4 additional burr holes (0.7 mm diameter) for EEG electrode placement. The EMG electrodes were then guided down the back of the neck underneath the trapezius muscle. EEG and EMG electrodes and optical fibers were glued into place using a mixture of dental cement and cyanoacrylate glue to provide insulation and structural stability. The optical fibers were manufactured in-house by assembling a fiber optic cable (200 μm outer diameter, ThorLabs, Cat. #FT200EMT) inserted into a ferrule (ceramic, 200 µm internal diameter, ThorLabs, Cat. CFLC230-10) and epoxied into place (Precision Fiber Products, Chula Vista, CA, Cat. #353ND). The optical fiber was cut to size (5.5 mm) and then flat cleaved and polished at the mating end of the ferrule. Sleep-wake monitoring, signal processing, optogenetic experiments and immunohistochemistry Sleep-wake recordings were conducted 2 weeks after surgeries. For recordings the mice were housed individually in transparent barrels in an insulated sound-proofed recording chamber maintained at an ambient temperature of 22 ± 1 °C and on a 12 h light/dark cycle (lights-on at 6 AM, Zeitgeber time: ZT0) with food and water available ad libitum . Mice were habituated for at least 3 days before commencing polysomnographic recordings. Cortical EEG (ipsilateral frontoparietal leads) and EMG signals were amplified x5000 (Model 3600; AM Systems, Sequim, WA) and digitized with a resolution of 500 Hz using a Micro 1401-3 (Cambridge Electronic Design; Cambridge, UK). Offline, EEG signals were digitally filtered using a 2 nd order Butterworth, band-pass, zero-phase filter with cut-off frequencies 0.5 Hz and 225 Hz filtfilt function, MATLAB (version R2020B; Mathworks, Natick, MA). EMG signals were likewise filtered using cut-off frequencies 100 Hz and 225 Hz. Also, for the trial-averaged analysis of EMG responses to light stimulation, EMG time series were integrated, smoothed (MATLAB; smooth function; 500-sample window), and normalized according to the pre-stimulus mean. Continuous wavelet transform of EEG signals were performed using MATLAB based tools developed by Grinsted and colleges (Available for download at: https://github.com/grinsted/wavelet-coherence ). For optogenetic experiments, experiments were carried out between ZT3-ZT9 (a period of low activity in nocturnal mice). We modified an open-source Online Sleep Detection script (Spike 2, Cambridge Electronic Design, source code available from the Cambridge Electronic Design website) to detect when mice had been in NREM sleep or REM sleep for at least 20 s, to trigger a 12-15 mW, 473 nm blue light (R471003GX, LaserGlow, Toronto, Canada) stimulation to the VLPO. The stimulation consisted of light pulses (5 ms) delivered at frequencies 1, 5, 10, 20 Hz over a 10 s period, delivered in random order throughout the recording session. A refractory period of at least 3 min was allowed between each stimulation, no mouse received more than 200 stimulations over any recording session and each recording session was separated by at least two days. Following the recordings, we intracardially perfused the mice with formalin (10% buffered solution) under deep anesthesia with isoflurane (5% in O 2 ). Brains were post-fixed in formalin (10% buffered solution, overnight), cryoprotected (20% sucrose), and cut into 40 μm sections. To verify the location of AAV-DIO-ChR2-mCherry injections sites, we incubated the sections in rabbit anti-ds Red primary antibodies (1:3000: overnight; Cat. #: 632496; Lot #: 1904182; Takara Bio USA, Mountain View, CA) and then in Alexa Fluor-555-conjugated donkey anti-rabbit secondary antibodies (1:500; Cat. #: A31572; Lot #: 2286312; 2hr; Invitrogen). We mapped the distribution of the ChR2- mCherry expressing neurons for each recorded animal as described in the methods above. No ChR2-mCherry expression was found in WT mice ( n = 3). Sleep scoring, analysis and statistics We used a custom-written MATLAB script for scoring arousals within stimulation periods on a trial-by-trial basis. The scorer was presented with a 30 s epoch of EEG and EMG recording centered on the stimulation period. The scorer was blinded to the animal genotype and stimulation condition (i.e., sham versus 1, 5, 10, or 20 Hz). The scorer determined, through visual inspection, if arousal occurred within the 10s-long stimulation period. Scored arousals required an EEG change lasting at least three seconds. We excluded trials where the 10 s pre-stimulus period contained a mixture of states (e.g., micro-arousals, muscle twitching activity, NREM-to-REM transitionary states). Sham stimulation trials were interleaved amongst the real laser stimulations. To examine the time course of evoked EEG and EMG responses to light stimulation, we computed the continuous wavelet transform of the EEG and the integral of the EMG for each stimulation trial, inclusive of the 10 s before and the 20 s after the stimulation period. Mean EEG wavelet power and integrated EMG signals from each animal were subsequently averaged ( n = 5). For the mean EMG signal we calculated the bootstrap confidence interval (MATLAB; bootci function). For average EEG power plots, confidence interval contours were computed as follows. For each animal we calculated the difference in wavelet power (real minus sham) across the time-frequency plane ((−10 to +30 s) x (0.5–30 Hz)). The data was smoothed in the time-domain (500-sample-wide moving average) and were subsequently down-sampled by a factor of 10. We used bootstrap resampling, with replacement, of the paired difference plots (all 3,125 permutations) to calculate the 95% bootstrap confidence interval of the mean power difference at each time-frequency coordinate. 5% significance contours were drawn around regions in the spectral plane where effect size confidence intervals excluded zero. Very small clusters of significance were removed for clarity and statistical conservatism. All parametric statistical testing were carried out using Sigmastat (version 4.0, Systat Software Inc. San Jose, CA). Paired bootstrap resampling was performed using MATLAB; in each case, 5000 bootstrap samples were taken, and confidence intervals were bias-corrected and accelerated. The details of the statistical tests used for each experiment may be found in the results. Effect sizes were considered statistically significant for p <  0.05. All experimental data were subject to histological validation. Data were excluded if the conditions of the histological validation were not met (i.e., cases in which there was not adequate bilateral transduction of the viral vector or optical fiber placement was not correctly positioned). All behavioral recordings were scored by an investigator that was blinded to the recording conditions. We represented data as mean ± SEM and n refers to the number of animals per group. Brain slice preparations and in vitro electrophysiological recordings We deeply anesthetized mice with isoflurane via inhalation (5% in O2) and transcardially perfused them with ice-cold modified ACSF (N-Methyl-D-glucamin- (NMDG)-based ACSF solution). We quickly removed the mouse brains and sectioned them in coronal slices (250 µm-thickness) in ice-cold NMDG-based ACSF using a vibrating microtome (VT1200S, Leica, Bannockburn, IL). We incubated the recording slices first for 5 min at 37 °C in NMDG-based ACSF, then in normal ACSF (Na-based solution) for an additional 10 min at 37 °C, and then we let them return to room temperature (RT) for at least 1 h. We recorded VLPO neurons in brain slices submerged and perfused (1–1.5 ml/min) with Na-based ACSF. We recorded under infrared differential interference contrast (IR-DIC) visualization and we recorded fluorescently labeled neurons using a combination of fluorescence and IR-DIC microscopy. We used a fixed-stage upright microscope (BX51WI, Olympus America Inc.) equipped with a Nomarski water immersion lens (Olympus 40X/0.8NAW) and an IR-sensitive CCD camera (ORCA-ER, Hamamatsu, Bridgewater, NJ). Real-time images were acquired using MATLAB (MathWorks) script software. We recorded VLPO neurons in whole-cell and cell-attached configurations using a Multiclamp 700B amplifier (Molecular Devices, Foster City, CA), a Digidata 1322 A interface, and Clampex 9.0 software (Molecular Devices). Neurons showing changes in input resistance of more than 10% over time, were excluded from the analysis. We recorded action potential firing in Na-based ACSF in cell-attached (voltage-clamp mode; Vh = 0 mV) or in whole-cell (current-clamp mode) configurations using the K-gluconate-based solution. For cells that were not spontaneously active we raised the ACSF KCl concentration from 2.5 to 6.3 mM. For the CRACM experiments we photostimulate ChR2 expressing neurons, axons, and terminals in VLPO using full-field light pulses (~10 mW/mm 2 , 1 mm beam width) from a 5 W Luxeon blue light-emitting diode (470 nm wavelength; Thorlabs, Newton, NJ; Cat. #M470L2-C4) coupled to epifluorescence pathway of microscope. We photostimulated with 10 ms light pulses (0.1 Hz, for a minimum of 30 trials). In some recordings, we used 60 s trains at 10 and 20 Hz (10 ms light pulses). We recorded spontaneous inhibitory postsynaptic currents (sIPSCs) and opto- evoked IPSCs (oIPSCs) in Na-based ACSF using a Cs-methane-sulfonate-based pipette solution at Vh = 0 mV. We recorded VLPO GABA/Gal neurons while photostimulating the local VLPO GABA/Gal →VLPO GABA/Gal and VLPO GABA → VLPO GABA/Gal inputs at the reversal potential of the ChR2-mediated current [19] , [20] determined for each cell (Vh = −5 to −15 mV) . We recorded opto-evoked excitatory postsynaptic currents (oEPSCs) in Na-based ACSF ( V h = −70 mV) using the K-gluconate-based pipette solution. In all the recordings we added 0.5% biocytin in the pipette solutions to mark the recorded neurons. Solutions and Chemicals The NMDG-based ACSF contained (in mM): 100 NMDG, 2.5 KCl, 1.24 NaH 2 PO 4 , 30 NaHCO 3 , 25 glucose, 20 HEPES, 2 thiourea, 5 Na-L-ascorbate, 3 Na-pyruvate, 0.5 CaCl 2 , 10 MgSO 4 (pH 7.3 with HCl with 95% O 2 and 5% CO 2 ; 310–320 mOsm). The Na-based-ACSF contained (in mM): 120 NaCl, 2.5 KCl, 1.3 MgCl 2 , 10 glucose, 26 NaHCO 3 , 1.24 NaH 2 PO 4 , 4 CaCl 2 , 2 thiourea, 1 Na-L-ascorbate, 3 Na-pyruvate (pH 7.3–7.4 with 95% O 2 and 5% CO 2 ; 310–320 mOsm). The K-gluconate-based solution contained (in mM): 120 K-Gluconate, 10 KCl, 3 MgCl 2 , 10 HEPES, 2.5 K-ATP, 0.5 Na-GTP (pH 7.2 adjusted with KOH; 280 mOsm). The Cs-methane-sulfonate-based pipette solution contained (in mM): 125 Cs-methane-sulfonate, 11 KCl, 10 HEPES, 0.1 CaCl 2 , 1 EGTA, 5 Mg-ATP and 0.3 Na-GTP (pH 7.2 adjusted with CsOH, 280 mOsm). We purchased Ox-A from Bachem (Bubendorf, Switzerland), noradrenalin, tetrodotoxin, and kynurenic acid from Cayman Chemical (Ann Arbor, MI), carbachol, bicuculline methiodide from Tocris Bioscience (Ellisville, MO). We purchased all other chemicals from Fisher Scientific (Waltham, MA) or Sigma-Aldrich (Saint Luis, MO). Data analysis and statistics for in vitro recordings We analyzed recording data using Clampfit 10 (Molecular Devices), MiniAnalysis 6 (Synaptosoft, Leonia, NJ), Python 3 ( www.python.org ) and MATLAB (version R2020B; MathWorks) software. We prepared the figures using Igor Pro 6 (WaveMetrics), Prism 7 (GraphPad, La Jolla, CA), Inkscape (GitLab), Photoshop (Adobe), and BioRender software. To ensure unbiased detection of the synaptic events, IPSCs and EPSCs were detected and analyzed automatically using MiniAnalysis. We measured synaptic event frequency and amplitude in control ACSF (last 5 min before drug applications), drug application (last 5 min of 10–15 min of drug applications), and in washout (last 5 min of 30–40 min washouts). We used the nonparametric Kolmogorov-Smirnov test (K-S test; MiniAnalysis) to evaluate the responses of drugs on sIPSC frequency or amplitude (statistical significance for p < 0.05, K-S test). We statistically compared mean sIPSC inter-event interval cumulative distributions using two-way repeated-measures (RM) ANOVA followed by Bonferroni’s multiple comparisons post-hoc test. We considered VLPO neurons to be responsive to photostimulation if the oEPSC or oIPSC probability during the first 50 ms that follows the light pulses was greater than baseline EPSC/IPSC probability + five times the SEM (baseline EPSC probability = 22.43 ± 1.84%, n = 61; baseline IPSC probability = 9.08 ± 1.83, n = 14) [23] . We calculated the latency of the oEPSCs and oIPSCs as the time difference between the start of the light pulse and the 5% rise point of the first synaptic event [48] . We calculated firing frequency and membrane potential changes by comparing values in control ACSF (last 2 min before drug applications), drug application (last 2 min of the 4–6 min of drug applications), and in washout (last 2 min of the 15–20 min washout). We represented data as mean ± SEM and n refers to the number of cells per group, unless otherwise specified. We compared group means using one-way or two-way RM ANOVA followed by Bonferroni’s multiple comparisons post-hoc test ( adjusted-p-value, adj-p ) or paired t -tests. Values showing p < 0.05 were considered significant. Peak-scaled non-stationary fluctuation analysis We used peak-scaled non-stationary fluctuation analysis to determine changes in GABA A single-channel current ( i ) or in the number of GABA A channels activated ( N ) in response to Ox-A [21] , [22] , [23] , [49] . As previously described [23] , we low-pass filtered and then aligned the peaks of photo-evoked IPSCs. We scaled the averaged mean-current waveform to the peak amplitude of individual oIPSCs, squared the difference, and then sampled this variance time series in 30 bins of equal current decrement from peak to baseline. The binned variance, was plotted against the mean-current amplitude (Fig. 4j ). We estimated the N and the i values by least-squares fitting of the peak-scaled variance and mean-current curve to the equation: δ 2 = iI–I 2 /N + b where δ 2 is the variance, I is the mean-current, and b is baseline variance. For each cell, we selected a minimum of 20 oIPSCs that had no overlapping spontaneous IPSCs. All the analysis was done using software written in Python 3. Immunohistochemistry, in situ hybridization and RNA scope in situ hybridization Following recordings, we fixed the recorded and adjacent slices, and the block of brain containing the AAV injection sites in formalin (10% buffered solution, overnight). The blocks containing the injection sites were then cryoprotected (20% sucrose) and recut in 40 µm sections with a sliding microtome (Microm HM 440E, GMI Inc., Minneapolis, MN). We processed the recorded slices with streptavidin-conjugated Alexa Fluor-488 (green; 1:500; Cat#: S32354 and Lot#: 1719656) or Alexa Fluor-555 (orange-red; 1:500; Cat#: S21381 and Lot#: 1010095; overnight; Invitrogen, Thermo Fisher Scientific Waltham, MA; Fig. 2 , Supplementary Figs. 4 and 6 ). We imaged the recorded fluorescently labeled neurons using a confocal microscope (Zeiss, LSM 5 Pascal) and Zen 2009 software (Zeiss) and we mapped their distribution onto template drawings [50] . We mapped the distribution of the ChR2-mCherry and ChR2-eYFP expressing neurons for each recorded animal by enhancing mCherry and YFP fluorescence by immunolabeling. For ChR2-mCherry immunolabeling we used rabbit anti-ds Red primary antibodies (1:3000; overnight; Cat. #: 632496; Lot #: 1904182; Takara Bio USA) and Alexa Fluor-555-conjugated donkey anti-rabbit secondary antibodies (1:500; Cat. #: A31572; Lot #: 2286312; overnight; Invitrogen). For ChR2-eYFP immunolabeling we used chicken anti-GFP primary antibodies (1:2000; overnight; Cat. #: A10262; Lot #: 2156242; Invitrogen) and Alexa Fluor-488-conjugated goat anti-chicken secondary antibodies (1:500; Cat. #: A11039; Lot #: 2304258; overnight; Invitrogen). We wet mounted and we scanned the whole sections using a slide scanner (Olympus VS120) or a confocal microscope (Zeiss LSM 5 Pascal) at a final magnification of 20X. We used a z-stack at 3–8 µm intervals to image throughout the slice. We viewed stacks of images using OlyVIA (Olympus) or Zen 2009 (Zeiss) software to identify the region containing transduced somata. We plotted the outline regions containing ChR2-mCherry or ChR2-eYFP labelled neurons onto template drawings [50] using Photoshop (Adobe). We compiled the distribution of ChR2-mCherry or ChR2-eYFP expressing neurons in a color map using a Python script [51] , representing the region of maximum number of overlapping cases in deep red, with the hues to green, light blue, to deep blue indicating fewer (Fig. 4 and Fig. 6 ). We validated the AAV-DIO-ChR2-mCherry and the AAV-DIO-ChR2-eYFP in Ox-IRES-Cre mice by immunolabeling. We processed for Ox immunoreactivity slices from Ox-IRES-Cre mice that were injected in the lateral hypothalamus with AAV-DIO-ChR2- mCherry ( n = 2 mice) and AAV-DIO-ChR2-eYFP ( n = 2 mice; Fig. 1 and Supplementary Table 1 ). Sections (40 μm) were only processed for immunohistochemistry for Ox whereas mCherry native fluorescence was used for the ChR2-mCherry labelling. We incubated the sections in goat anti-Ox-A (1:500; Cat. #: sc-8070; Lot #: A2915; Santa Cruz Biotechnology, Dallas, TX) primary antibodies (overnight) and then in Alexa Fluor-488-conjugated donkey anti-goat (1:500, Cat. #: A11055; Lot #: 1942238; Invitrogen) secondary antibodies (2 h) [23] . Sections from mice injected with AAV-DIO-ChR2-eYFP were processed for immunohistochemistry for both Ox and YFP. We incubated the sections in goat anti-Ox-A (1:500; Cat. #: sc-8070; Lot #: A2915; Santa Cruz Biotechnology) and chicken anti-GFP (1:2000; Cat. #: A10262; Lot #: 2156242; Invitrogen) primary antibodies (overnight) and then in Alexa Fluor-555-conjugated donkey anti-goat (1:500; Cat. #: A21432; Lot #: 1697092; Invitrogen) and Alexa Fluor-488-conjugated rabbit anti-chicken (1:500; Cat. #: NB710-94968; Lot #: 143-090; Novus Biologicals, Littleton, CO) secondary antibodies (2 hr). We counted the ChR2-mCherry expressing neurons (native fluorescence) and the ChR2-eYFP expressing neurons (immunolabeled in green with Alexa-Fluor-488) that were double-labeled for Ox immunoreactivity using a confocal microscope (Zeiss LSM 5 Pascal) and Zen 2009 software (Zeiss). To visualize the Ox innervation of VLPO we processed for Ox immunolabeling sections from WT mice ( n = 4 mice). We intracardially perfused the mice with formalin (10% buffered solution) under deep anesthesia with isoflurane (5% in O 2 ) . Brains are post-fixed in formalin (10% buffered solution, overnight), cryoprotected (20% sucrose), and cut into 40 μm sections into 3 series using a sliding microtome (Microm HM 440E, GMI Inc., Minneapolis, MN). We incubated the sections in goat anti-Ox-A (1:500; Cat. #: sc-8070; Lot #: A2915; Santa Cruz Biotechnology) primary antibodies (overnight) and then in Alexa Fluor-555-conjugated donkey anti-goat (1:500; Cat. #: A21432; Lot #: 1697092; Invitrogen) secondary antibodies (2 h) [23] . We imaged and photographed the covered sections (Vectashield mounting medium; Vector Laboratories, San Diego, CA) visualized and photographed the sections using a confocal microscope (Zeiss LSM 5 Pascal), and Zen 2009 software (Zeiss). We performed DIG-labeled RNA probe in situ hybridization for Vgat ( Slc32a1 ) mRNA in Vgat-IRES-Cre mice injected into the VLPO with AAV-DIO-TdTomato ( n = 2 mice) or with AAV-DIO-GFP ( n = 2 mice) (Supplementary Fig. 5 and Supplementary Table 1 ) [23] . Four weeks after AAV injections, we intracardially perfused the mice with formalin (10% buffered solution) under deep anesthesia with isoflurane (5% in O 2 ). Brains were post-fixed in formalin (10% buffered solution, overnight), cryoprotected (20% sucrose), and cut into 40 μm sections into 3 series using a sliding microtome (Microm HM 440E, GMI Inc). Sections were washed in RNAse-free PBS, containing diethylpyrocarbonate (DEPC) and then incubated in hybridization buffer at 53 ˚C (1 h). The Vgat probe was denatured at 80˚C (10 min) and then added to the hybridization buffer and incubated overnight at 53 ˚C. The sections were washed in saline citrate (SSC) with 50% formamide at 53 ˚C (2 h), washed in tris buffered saline (TBS; pH 7.5; 30 min), incubated in 1% blocking reagent (Roche Applied Science, Penzberg, Germany; 30 min), incubated in peroxidase-conjugated DIG antibodies (1:500, Cat. #: 11207733910; Lot #: 13296300; Roche Applied Science, now Millipore Sigma; overnight) and then washed in TBS. Sections from mice injected with AAV-DIO-GFP were labeled with Cy3 (red) by Tyramide signal amplification (1:50, Perkin Elmer, Waltham, MA; 30 min) then immunolabeled for GFP with chicken anti-GFP primary antibodies (1:2000; Cat. #: A10262; Lot #: 2156242; Invitrogen; overnight) and then in Alexa Fluor-488-conjugated goat anti-chicken secondary antibodies (1:500; Cat. #: A11039; Lot #: 2304258; Invitrogen; 2 h). Sections from mice injected with AAV-DIO-TdTomato were labeled with Cy5 (far-red) by Tyramide signal amplification (1:50, Perkin Elmer; 30 min) then immunolabeled for TdTomato with rabbit anti-ds Red primary antibodies (1:500, Cat. #: 632496; Lot #: 1904182; Takara Bio USA; overnight) and then in Alexa Fluor-555-conjugated donkey anti- rabbit secondary antibodies (1:500, Cat. #: A31572; Lot #: 2286312; Invitrogen; 2 hr). Sections were washed first in TBS and then in PBS, mounted, and coverslipped in deionized water. We imaged and photographed the sections using a confocal microscope (Zeiss LSM 5 Pascal). The Vgat probe was provided by Dr. Shigefumi Yokota (University School of Medicine, Izumo, Japan) [23] . For RNA scope in situ hybridization for Gal , Vgat and Hcrtr2 mRNAs, we used RNA Scope Multiplex Fluorescent Reagent Kit V2 Advanced Cell Diagnostics, Hayward, CA; Cat. #323100. We intracardially perfused the mice with formalin (10% buffered solution) under deep anesthesia with isoflurane (5% in O 2 ). Brains were post-fixed in formalin (10% buffered solution, overnight), cryoprotected (20% sucrose), and cut into 30 μm sections. The sections were treated with hydrogen peroxide (20 min; RT). We then performed a target retrieval procedure at 100 ˚C (5 min), treated the sections with protease (40 ˚C; 30 min; Protease III, RNA scope) and incubated them with RNA scope probes for galanin -C1 (RNA scope® Probe- Mm- Gal ; Cat. #400961), Vgat -C2 (RNA scope® Probe- Mm- Slc32a1 ; Cat. #319199) and Hcrtr2 -C3 (RNA scope® Probe- Mm- Hcrtr2-O1 ; Advanced Cell Diagnostics; Cat. #581631) for the hybridization step (2 hr; 40 °C). After hybridization, we performed the amplification steps (40 °C; AMP1-FL and AMP2-FL: 30 min each; AMP3-FL: 15 min), followed by horse radish peroxidase-C1 (HRP-C1) amplification (40 °C for 15 min). Sections were then incubated in TSA plus Cy3 (Perkin Elmer; Cat. #NEL744001KT) to visualize Gal (Channel 1 at 550 nm) mRNA in red. This is followed by incubating the sections in HRP-C2 amplification step (40 °C; 15 min). Sections were then incubated in TSA plus Fluorescein (Perkin Elmer, Cat. #: NEL754001KT) fluorophore (1:1000; 30 min) to visualize Vgat (Channel 2 at 488 nm) in green. In the last step of the process, sections were subjected to HRP-C3 amplification (40 °C; 15 min) followed by TSA plus Cy5 incubation (40 °C; 30 min; Perkin Elmer; Cat. #NEL754001KT) to visualize Hcrtr2 (Channel 3 at 647 nm) mRNA in magenta. After each fluorophore step, sections were subjected to HRP blocking (40 °C; 15 min). After each step in the protocol, we washed the sections two times with 1X wash buffer provided in the kit. We combined RNA scope in situ hybridization for Vgat mRNA (in Vgat-Flp mice) and for Gal mRNA (in Gal-IRES-Cre mice) with immunolabeling for YFP and TdTomato (Supplementary Fig. 8 and Supplementary Table 1 ). Mice were injected into the VLPO with AAV-fDIO-ChR2-eYFP ( n = 2 Vgat-Flp mice) or with AAV-DIO-TdTomato ( n = 2 Gal-IRES-Cre mice). Four weeks after AAV injections, we intracardially perfused the mice with formalin (10% buffered solution) under deep anesthesia with isoflurane (5% in O 2 ). Brains were post-fixed in formalin (10% buffered solution, overnight), cryoprotected (20% sucrose) and cut into 30 μm, and processed for RNA scope in situ hybridization for Vgat mRNA following the protocol described above. For the sections from Vgat-Flp mice injected with AAV-fDIO-ChR2-eYFP the Vgat mRNA was labeled with Cy3 (in red) and then the sections were immunolabeled for GFP (in green) with chicken anti-GFP primary antibodies (1:2000; Cat. #: A10262; Lot #: 2156242; Invitrogen; over 2 nights) and then in Alexa Fluor-488-conjugated goat anti-chicken secondary antibodies (1:500; Cat. #: A11039; Lot #: 2304258; Invitrogen; 4 hr). For the sections from Gal-IRES-Cre mice injected with AAV-DIO-TdTomato the Gal mRNA was labeled with Fluorescein fluorophore (in green) and then the sections were immunolabeled for TdTomato with rabbit anti-ds Red primary antibodies (1:1000, Cat. #: 632496; Lot #: 1904182; Takara Bio USA; over 2 nights) and then in Alexa Fluor-555-conjugated donkey anti-rabbit secondary antibodies (1:500; Cat. #: A31572; Lot #: 2286312; Invitrogen; 4 hr). We imaged and photographed the covered sections (Vectashield mounting medium; Vector Laboratories) with a confocal microscope (Leica Stellaris 5) at final magnification of 20X and 63X. We used a z-stack at 3–5 µm intervals to image throughout the slice after tile acquisition. We viewed stacks of images using image J software to identify the region containing the VLPO and the fluorescent signals for RNA scope and immunohistochemistry at cellular level. Single cell RT-PCR and RT-sqPCR To identify the phenotype of recorded neurons, we performed single-cell reverse transcription-polymerase chain reaction (scRT-PCR) and semi-quantitative scRT-PCR (scRT-sqPCR). After completing whole-cell recordings, we harvested the cytoplasm of the recorded VLPO neurons ( n = 26) through aspiration controlled under fluorescent and IR-DIC visualizations. We then performed cDNA synthesis as previously described [52] using the single-cell-to-CT TM kit (Ambion, Thermo Fisher Scientific). We first converted the mRNA into cDNA (9 µl of Single Cell Lysis buffer and 1 µl of DNAase I solution to each extracted sample stored in RNAse-free PCR tubes; room temperature; 5 min), stopped the reaction (1 µl of Stop solution; room temperature; 2 min) and stored the samples (−20 °C; up to two months). For the pre-amplification protocol, we added 3 µl VILO and 1.5 µl Cell Superscript to each sample (25 °C; 10 min; 42 °C; 60 min and 85 °C; 5 min). We then added (PreAmp Mix 5 µl and of Taqman Gene Expression Master mix 6 µl to each sample; 95 °C; 10 min). We repeated 14 cycles (95 °C; 15 s and 60 °C; 4 min). Samples were then processed for scRT-PCR or scRT-sqPCR. For scRT-PCR, amplification of cDNA encoding for the galanin ( Gal ), glyceraldehyde 3-phosphate dehydrogenase ( Gapdh ), glutamate decarboxylase Gad2 (Gad65) and Gad1 (Gad67) were performed in two rounds amplifications (40 cycles each). For the second amplification we used a 1:6 dilution of the first amplification material. Gal 1 st amplification primers: Gal F: 5′-GGCTGGCTCCTGTTGGTTGT-3′ and Gal R: 5′- GCTCTCAGGCAGGGGCAC-3′ (annealing temperature; AT: 57.2 °C; expected amplimer size: 228 base pair, bp). Gal 2 nd amplification primers: Gal 2F: 5′- TCTGGGACTTGGGATGCCTG-3′ and Gal 2R: 5′-GGGGCACATCAACACTTCCT-3′ (AT: 54.1 °C; expected amplimer size: 182 bp) [18] . Gapdh 1 st amplification primers: Gapdh F: 5′-AACTTTGGCATTGTGGAAGG-3′ and Gapdh R: 5′-TGTGAGGGAGATGCTCAGTG-3′ (AT: 61.8 °C; expected amplimer size: 600 bp). Gapdh 2 nd amplification primers: Gapdh 2F: 5′-ACCCAGAAGACTGTGGATGG-3′ and Gapdh 2R: 5′-CACATTGGGGGTAGGAACAC-3′ (AT: 63.2 °C; expected amplimer size: 171 bp). Gad2 1 st amplification primers: Gad2 F: 5′-CCAAAAGTTCACGGGCGG-3′ and Gad2 R: 5′- TCCTCCAGATTTTGCGGTTG-3′ (AT: 52 °C; expected amplimer size: 375 bp). Gad2 2 nd amplification primers: Gad2 2F: 5′-CACCTGCGACCAAAAACCCT-3′ and Gad2 2R: 5′-GATTTTGCGGTTGGTCTGCC-3′ (AT: 54.2 °C; expected amplimer size: 248 bp). Gad1 1 st amplification primers: Gad1 F: 5′-ATGATACTTGGTGTGGCGTAGC-3′ and Gad1 R: 5′- GTTTGCTCCTCCCCGTTCTTAG-3′ (AT: 65 °C; expected amplimer size: 253 bp). Gad1 2 nd amplification primers: Gad1 2F: 5′-CAATAGCCTGGAAGAGAAGAGTC-3′ and Gad1 2 R: 5′-GTTTGCTCCTCCCCGTTCTTAG G-3′ (AT: 63 °C; expected amplimer size: 177 bp) [18] . First and second amplification reactions were conducted mixing (4 µl of first-strand cDNA template or pre-amplified, 10 µl reaction mix REDExtract-N-Amp PCR ReadyMix; Sigma-Aldrich and 0.4 µl for each primer; 0.2 to 0.4 µM). The final reaction volume was adjusted to 20 µl with nuclease-free water (Ambion, Thermo Fisher Scientific). Products were visualized by staining with ethidium bromide (Invitrogen) and analyzed by electrophoresis in 1.5-2% agarose gels. We used Primer 3web 4.1.0 software ( http://primer3.wi.mit.edu/ ) to verify the Gal , Gapdh , Gad1 , and Gad2 primers. The sequencing of the second amplification samples that contain the Gal , Gapdh , Gad2 and Gad1 amplicons were conducted by Quintara Bioscience (Boston, MA). We verified the sequence results to the Gal , Gapdh , Gad2 and Gad1 sequences (NCBI GenBank) using Genetyx software. Molecular identification was based on the results from the second reaction. We purchased all the custom primers from Sigma-Aldrich, St. Louis, MO. For scRT-sqPCR, the cDNAs ( n = 38 neurons) were produced as described in the section above. We performed TaqMan™ based probe assay for semi-quantitative gene expressions using the 7500 Fast Real-Time PCR (Applied Biosystems; Foster City, CA). We added cDNA template (2.5–3 µl) enzyme master mix (12.5 µl; TaqMan Universal PCR Master Mix, Applied Biosystems) and TaqMan Gene Expression assays for the amplification of Gal and Gapdh cDNAs (1.25 µl; ThermoFisher Scientific). Volumes for the reactions were adjusted to 25  µl with H 2 O. The Gal cDNA probe was tagged to FAM/MGB and the Gapdh cDNA to VIC/MGB. TaqMan TM Gene Expression assays for the Gal cDNA (TaqMan Assay Reagents, Gal , 20X, Cat. #4331182) and for Gapdh cDNA (Pre- Developed Gapdh TaqMan Assay Reagents, 20X, Cat. #4352339E). The thermal cycling conditions were as follows: enzyme activation (95 °C; 10 min), followed by DNA denaturation (95 °C; 15 s; 45–50 cycles) and annealing/extension (60 °C; 1 min). Relative gene expression between samples was calculated using the 2 -Ct method [53] , [54] . Data were normalized to the Gapdh expression levels. As control group, we used TdTomato labeled VLPO GABA/Gal neurons. We used values of 50 for non-detects Ct. Each sample was run in duplicates (2 times, in 2 separate reactions). We considered scRT-PCR- and scRT- sqPCR-negative, samples in which Gapdh expression was undetectable. We represented data as mean ± SEM and n refers to the number of cells per group and we compared group means using Mann-Whitney unpaired t-test. Single cell RNA sequencing data analysis Single cell RNA-sequencing (scRNA-seq) data of the POA [24] were retrieved from the Gene Expression Omnibus (GEO) repository (GSE113576). Data were available as unique Digital Gene Expression (DGE) matrix. Briefly, the DGE matrix was imported into R software (v.3.6.3) and all the downstream processing was performed using functionalities provided by the R library Seurat (Seurat v.3.1.5) [55] , [56] , [57] . Expression data were filtered according to the following criteria: (i) cells expressing >200 genes and with a mitochondrial gene expression rate <10% were retained; (ii) genes detected in >2 cells were retained. Seurat3 was used to cluster all POA cells and to perform Differential Gene Expression between clusters. Genes expressed only or expressed predominantly in a specific cluster were identified as marker genes. (Supplementary Fig. 9 , Supplementary Table 2 ). Afterwards, clusters corresponding to glial cell types were discarded and neuronal clusters were retained for downstream analyses. According to the spatial information gathered from Multiplexed Error-Robust Fluorescence In Situ Hybridization ( Multiplexed Error-Robust Fluorescence In Situ Hybridization ) [24] and in situ hybridization  from the Allen Brain Atlas, we isolated only neuronal clusters located in the VLPO (#i5, i8, i10, i20, i26, i29, i35, i37, i39, e3, e7, e11, e20 and e24). Briefly, the following Seurat v.3.1.5 functions were used: (1) SCTransform () to normalize and scale the data, to identify the top 3000 variable genes, and to correct for number of unique molecular identifiers (UMIs), percentage of mitochondrial gene expression, and difference between S and G2M cell cycle scores. Cell cycle scores were inferred using CellCycleScoring () function [58] ; (2) runPCA was used to calculate the first 50 Principal Components (PCs) of the 3000 most variable features; (3) FindNeighbors () to construct a Shared Nearest Neighbor (SNN) Graph. This method first determines the k-nearest neighbors (knn) of each cell and then uses this knn graph to construct the SNN graph by calculating the neighborhood overlap (Jaccard index) between every cell and its k.param nearest neighbors; (4) FindClusters to define the cell clusters and their granularity using the original Louvain algorithm at resolution of 0.6 for all cells and 1.2 for neurons; (5) runTSNE for t-Distributed Stochastic Neighbor Embedding (t-SNE) dimensional reduction method, to visualize cell clusters in 2 dimensions. (6) FindAllMarkers to perform a differential gene expression between each cluster versus all the other cells of the dataset using the non-parametric Wilcoxon Rank Sum statistics. A gene was defined as differentially expressed if absolute logFC was >0.25 and adjusted p-value ( adj-p ) (Bonferroni corrected) was <0.05. (7) finally, we used FindMarkers to compare two different cell clusters/groups. The abovementioned parameters were also applied to this function. Cells and neuronal clustering were performed using the same bioinformatic pipeline. Statistics and Reproducibility Figure 1a : an example of Ox innervation of the POA and VLPO by immunolabeling for Ox-A. The immunolabeling was conducted in n = 4 WT mice. Figure 1c an example of immunolabeling for ChR2-mCherry of n = 5 Ox-IRES-Cre mice used for whole-animal optogenetic studies. Figure 1d : an example of double labelling for ChR2-mCherry and Ox-A immunoreactivity to test selectivity of the AAV-DIO-ChR2-eYFP (and AAV-DIO-ChR2-mCherry ) for Ox neurons. Immunolabeling conducted in n = 4 Ox-IRES-Cre mice injected with AAV-DIO-ChR2-eYFP (and AAV-DIO-ChR2-mCherry ) into the Ox field. Figure 2a and b: map of n = 29 recorded neurons distributed in n = 19 slices from n = 14 WT mice. Figure 4a : an example of VLPO GABA neurons (in green) and VLPO GABA/Gal neurons (double-labeled in red and green) following the injection of a mix of AAV-fDIO-ChR2-eYFP and AAV-DIO-TdTomato into the VLPO of Vgat-Flp::Gal-IRES-Cre mice. This experiment was conducted in n = 10 Vgat-Flp::Gal-IRES-Cre mice. Figure 5e : an example of triple staining for Gal , Vgat ( Slc32a1 ) and Ox 2 R mRNAs by RNA scope in situ hybridization. This staining was conducted in n = 3 WT mice. Supplementary Fig. 4b : an example of double labeling for biocytin and TdTomato. This labelling was conducted in n = 3 recorded neurons distributed in n = 2 slices from n = 2 Vgat-IRES-Cre mice. Supplementary Fig. 5 : an example of double labelling for TdTomato (and AAV-DIO-GFP ) immunolabeling and Vgat mRNA in Vgat-IRES-Cre mice injected with AAV-DIO-TdTomato (and AAV-DIO-GFP ) into the VLPO. This labelling was conducted in n = 4 Vgat-IRES-Cre mice. Supplementary Fig. 6b : an example of double labeling for biocytin and TdTomato. This labelling was conducted in n = 3 recorded neurons distributed in n = 3 slices from n = 2 Gal-IRES-Cre mice. Supplementary Fig. 6c : an example of recordings from a TdTomato labeled VLPO GABA/Gal neurons. For these experiments we recorded from n = 49 labeled VLPO GABA/Gal neurons in n = 23 slices from n = 21 Gal-IRES-Cre mice. Supplementary Fig. 7a : an example of recordings from a TdTomato labeled VLPO GABA/Gal neurons. For these experiments we recorded from n = 9 labeled VLPO GABA/Gal neurons in n = 9 slices from n = 7 Gal-IRES-Cre mice. Supplementary Fig. 8a : an example of double labelling for ChR2-eYFP (immunolabeling) and Vgat mRNA in Vgat-Flp mice injected with AAV-fDIO-ChR2-eYFP into the VLPO. This labelling was conducted in n = 2 Vgat-Flp mice. Fig. 8b: an example of double labelling for TdTomato (immunolabeling) and Gal mRNA in Gal-IRES-Cre mice injected with AAV-DIO-TdTomato into the VLPO. This labelling was conducted in n = 2 Gal-IRES-Cre mice. Reporting summary Further information on research design is available in the Nature Research Reporting Summary linked to this article.